Dendritic cells induce Th2-mediated airway inflammatory responses to house dust mite via DNA-dependent protein kinase DNA-dependent protein kinase (DNA-PK) mediates double-stranded DNA break repair, V(D)J recombination and immunoglobulin class switch recombination, as well as innate immune and pro-inflammatory responses. However, there is limited information regarding the role of DNA-PK in adaptive immunity mediated by dendritic cells (DCs), which are the primary antigen-presenting cells in allergic asthma. Here we show that house dust mite induces DNA-PK phosphorylation, which is a marker of DNA-PK activation, in DCs via the generation of intracellular reactive oxygen species. We also demonstrate that pharmacological inhibition of DNA-PK, as well as the specific deletion of DNA-PK in DCs, attenuates the induction of allergic sensitization and Th2 immunity via a mechanism that involves the impaired presentation of mite antigens. Furthermore, pharmacological inhibition of DNA-PK following antigen priming similarly reduces the manifestations of mite-induced airway disease. Collectively, these findings suggest that DNA-PK may be a potential target for treatment of allergic asthma. DNA-dependent protein kinase (DNA-PK) is a key enzyme involved in the recognition and repair of double-stranded DNA breaks (DSB) by a process termed nonhomologous end-joining, whereby DNA ends are directly ligated [1] , [2] , [3] , [4] . This represents an important mechanism of cellular repair in response to DSB induced by ionizing radiation, as well as reactive oxygen species, that prevents chromosomal translocations and genetic instability that can lead to carcinogenesis or cellular death [2] , [5] . DNA-PK comprises a regulatory heterodimer of Ku proteins (Ku70 and Ku80) and a 465-kDa catalytic subunit, DNA-PKcs, which is a member of the phosphatidylinositol 3-kinase-related kinase family and functions as a serine/threonine kinase. DNA-PK also participates in additional processes that involve DSB repair, such as V(D)J recombination and class switch recombination [2] , [6] . Mice with the scid mutation affecting the Prkdc gene that encodes DNA-PKcs are unable to generate functional immunoglobulin and T-cell receptors and are deficient in mature B and T lymphocytes [7] , [8] , [9] , [10] . The scid missense mutation results in a premature stop codon that leads to diminished expression of the DNA-PKcs protein, and specifically impairs the differentiation of stem cells into mature lymphocytes, whereas myeloid differentiation is not affected [9] , [11] , [12] . Similarly, mice with a targeted disruption of the Prkdc gene, which encodes DNA-PKcs, have a phenotype of severe combined immunodeficiency (SCID) and radiosensitivity [13] . Although its canonical function is to mediate DSB repair by nonhomologous end-joining, DNA-PK has also been shown to regulate innate immune responses and pro-inflammatory signalling pathways [2] , [4] . For example, DNA-PK modulates host defense against viral infection by acting as a pattern recognition receptor that binds cytoplasmic DNA [14] . This activates an innate immune response mediated by type I interferons via a pathway involving IRF-3 (interferon regulatory factor 3), TANK-binding kinase 1 and stimulator of interferon genes. Interestingly, vaccinia virus has evolved a strategy to evade this mechanism [15] . The vaccinia virus C16 protein directly binds the Ku heterodimer, thereby blocking DNA-PK binding to DNA, which inhibits DNA sensing and innate immunity to DNA viruses. The mechanism of killing of CD4 + T cells during human immunodeficiency virus-1 (HIV-1) infection has also recently been shown to involve DNA-PK activation [16] . Integration of the HIV-1 genome into the host chromosome induces a double-stranded DNA damage response that activates DNA-PK and phosphorylates p53 and histone H2AX, with resultant death of CD4 + cells. Interestingly, HIV-1-mediated CD4 + cell death could be inhibited by pharmacological inhibitors of DNA-PK. Infection with Listeria monocytogenes also causes DNA-strand breaks that induce the phosphorylation and activation of DNA-PK, H2AX and CDC25A. This activates a DNA damage/replication checkpoint that delays cell cycle progression and thereby facilitates propagation of this intracellular pathogen [17] . DNA-PK also participates in an endosomal signalling pathway that induces a pro-inflammatory response in natural killer cells by phosphorylating Akt on Ser 473 (ref. 18 ). The DNA-PK-mediated phosphorylation of p50 NF-κB is similarly required for tumour necrosis factor-induced vascular cell adhesion protein 1 (VCAM-1) expression [19] . Lastly, DNA-PK mediates free fatty acid-induced lipid accumulation in hepatocytes, which may contribute to the pathogenesis of nonalcoholic steatohepatitis [20] . Since DNA-PK can regulate innate immunity and pro-inflammatory signalling pathways, we hypothesized that it might also modulate adaptive Th2-mediated immune responses to house dust mite (HDM) antigen. We also hypothesized that if DNA-PKs were involved in the pathogenesis of HDM-induced asthma, then pharmacological inhibitors of DNA-PK kinase activity might be utilized as a novel treatment approach. We focused on HDM because it is a clinically important aeroallergen that is a potent inducer of Th2-mediated immune responses and a common cause of allergic asthma worldwide. To investigate the role of DNA-PK in HDM-induced asthma, here we utilize genetic and pharmacological models, including the development of a CD11c-specific DNA-PKcs knockout mouse. We show that HDM activates DNA-PK in dendritic cells (DCs) via a reactive oxygen species (ROS)-dependent pathway. Furthermore, we show that DNA-PK is required for both effective antigen presentation by DCs, as well as the induction of HDM-induced Th2-mediated airway inflammation. This demonstrates a previously unidentified link between the role of DNA-PK in DCs and the induction of allergic sensitization and Th2 immunity in HDM-induced asthma. Furthermore, it identifies DNA-PK as a novel therapeutic target for the development of new treatments for asthmatic patients. HDM induces DNA-PK phosphorylation in DCs First, we considered whether HDM could induce the generation of intracellular ROS by human monocyte-derived DCs (moDCs) as a mechanism by which DNA-PK phosphorylation and activation are initiated. Stimulation of human moDCs with HDM induced the production of intracellular ROS, which could be inhibited by the antioxidant, NAC ( N -acetylcysteine), the NADPH oxidase/flavoprotein inhibitor, DPI (diphenyleneiodonium chloride) and the DNA-PK inhibitor, NU7441 ( Fig. 1a ) [21] . We then assessed whether human moDCs express DNA-PK and whether DNA-PK can be activated in response to HDM stimulation. Western blots of human moDC proteins demonstrated that DNA-PKcs is expressed under basal conditions and is activated in response to HDM stimulation, as evidenced by autophosphorylation on Ser 2056 , which is a marker of DNA-PK activity ( Fig. 1b ) [22] . DNA-PK activity peaks at 3 and 6 h and markedly diminishes by 24 h. HDM-induced DNA-PK phosphorylation at Ser 2056 at 6 h was inhibited by treatment with NU7441, as well as with NAC and DPI [21] . HDM stimulation also induced Akt phosphorylation on Ser 473 and Thr 308 that was maximal at 6 and 24 h. Levels of p-Akt (Ser 473 ) and p-Akt (Thr 308 ) were similarly reduced by NU7441, NAC and DPI. Collectively, these results demonstrate that HDM stimulates intracellular ROS generation by human moDCs and that ROS are required for the HDM-induced phosphorylation of DNA-PK, as well as Akt, which is downstream of DNA-PK signalling and has been reported to be a regulator of DC function [23] . 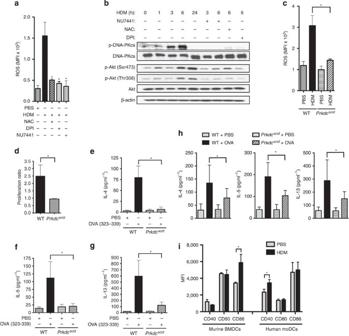Figure 1: HDM induces phosphorylation of DC DNA-PK via generation of ROS. (a) The MFI of intracellular ROS generated by human moDC stimulated with HDM (100 μg ml−1) for 1 h with or without NAC (2 mM), DPI (10 μM) or NU7441 (0.5 μM;n=3–5, *P<0.01 versus HDM, one-way analysis of variance (ANOVA) with Bonferroni multiple comparison test). (b) Western blots of HDM-stimulated human moDC proteins with or without NU7441, NAC or DPI for 1–24 h (seeSupplementary Fig. 2for images of full original blots). Image is representative of four blots. (c) MFI of intracellular ROS generated by BMDC from WT andPrkdcscidmice stimulated with HDM (100 μg ml ml−1) for 1 h (n=3, *P<0.01, WT+HDM versusPrkdcscid+HDM, one-way ANOVA with Bonferroni multiple comparison test). (d) CD11c+BMDC fromPrkdcscidand WT mice were pulsed with the OVA 323–339 peptide and incubated at a 1:5 ratio with CSFE-labelled CD4+DO11.10T cells for 4 days. OVA-specific proliferation is presented as the proliferation index (n=8, *P=0.0011, Mann–Whitney test, pooled data from three independent experiments). (e–g) Th2 cytokines released by co-cultures of OVA 323–329-pulsed BMDCs and CSFE-labelled DO11.10 CD3+/CD4+T cells (n=3, *P<0.05, WT+OVA versusPrkdcscid+OVA, one-way ANOVA with Bonferroni multiple comparison test). (h) Co-cultures of BMDCs fromPrkdcscidand WT mice incubated at a 1:5 ratio with splenic CD4+T cells from WT mice sensitized to full-length OVA. Co-cultures were treated with PBS or OVA (1 μg ml ml−1) for 4 days and Th2 cytokines were quantified (n=7, *P<0.05). Pooled data from two independent experiments. (i) MFI of CD40, CD80 and CD86 cell surface expression by murine BMDCs (n=6 mice) and human moDCs (n=10 mice) stimulated with or without HDM (100 μg ml−1) for 24 h. Pooled data from two independent experiments (*P<0.05, Mann–Whitney test). Figure 1: HDM induces phosphorylation of DC DNA-PK via generation of ROS. ( a ) The MFI of intracellular ROS generated by human moDC stimulated with HDM (100 μg ml −1 ) for 1 h with or without NAC (2 mM), DPI (10 μM) or NU7441 (0.5 μM; n =3–5, * P <0.01 versus HDM, one-way analysis of variance (ANOVA) with Bonferroni multiple comparison test). ( b ) Western blots of HDM-stimulated human moDC proteins with or without NU7441, NAC or DPI for 1–24 h (see Supplementary Fig. 2 for images of full original blots). Image is representative of four blots. ( c ) MFI of intracellular ROS generated by BMDC from WT and Prkdc scid mice stimulated with HDM (100 μg ml ml −1 ) for 1 h ( n =3, * P <0.01, WT+HDM versus Prkdc scid +HDM, one-way ANOVA with Bonferroni multiple comparison test). ( d ) CD11c + BMDC from Prkdc scid and WT mice were pulsed with the OVA 323–339 peptide and incubated at a 1:5 ratio with CSFE-labelled CD4 + DO11.10T cells for 4 days. OVA-specific proliferation is presented as the proliferation index ( n =8, * P =0.0011, Mann–Whitney test, pooled data from three independent experiments). ( e – g ) Th2 cytokines released by co-cultures of OVA 323–329-pulsed BMDCs and CSFE-labelled DO11.10 CD3 + /CD4 + T cells ( n =3, * P <0.05, WT+OVA versus Prkdc scid +OVA, one-way ANOVA with Bonferroni multiple comparison test). ( h ) Co-cultures of BMDCs from Prkdc scid and WT mice incubated at a 1:5 ratio with splenic CD4 + T cells from WT mice sensitized to full-length OVA. Co-cultures were treated with PBS or OVA (1 μg ml ml −1 ) for 4 days and Th2 cytokines were quantified ( n =7, * P <0.05). Pooled data from two independent experiments. ( i ) MFI of CD40, CD80 and CD86 cell surface expression by murine BMDCs ( n =6 mice) and human moDCs ( n =10 mice) stimulated with or without HDM (100 μg ml −1 ) for 24 h. Pooled data from two independent experiments (* P <0.05, Mann–Whitney test). Full size image Experiments were next performed with bone marrow-derived DCs (BMDCs) from Prkdc scid mice that have a spontaneous mutation in the Prkdc gene. HDM-challenged BMDCs from wild-type (WT), but not Prkdc scid mice, had increases in intracellular ROS generation ( Fig. 1c ). Thus, in addition to being activated by ROS, DNA-PK is required for HDM-induced ROS production by BMDCs. Next, BMDCs from Prkdc scid mice were used to investigate the role of DNA-PK in antigen-specific T-cell proliferation and Th2 cytokine production. Co-culture experiments of splenic CD4 + T cells from mice expressing the major histocompatibility complex II (MHCII)-restricted DO11.10T-cell receptor that recognizes the OVA 323–339 peptide showed that BMDCs from Prkdc scid mice have a reduced ability to induce both T-cell proliferation and Th2 cytokine production as compared with BMDCs from WT mice following ex vivo stimulation with the OVA 323–339 peptide ( Fig. 1d–g ) [24] . Similarly, BMDCs from Prkdc scid mice had an impaired ability to induce Th2 cytokine production following ex vivo stimulation with full-length ovalbumin (OVA) when co-cultured with splenic T cells from OVA-sensitized mice. Collectively, this shows that DNA-PK-deficient DCs have a primary defect in antigen presentation to T cells and are unable to mediate the antigen-specific production of Th2 effector cytokines. Lastly, we show that both murine BMDCs and human moDCs express the co-stimulatory molecules, CD40, CD80 and CD86 ( Fig. 1h ). Furthermore, HDM stimulation increased expression of CD86 by murine BMDCs and CD40 by human moDCs. DCs from Prkdc scid mice mediate reduced Th2 inflammation Adoptive transfer experiments using HDM-pulsed CD11c + BMDCs from WT and Prkdc scid mice were next utilized to define the role of DC DNA-PK in inducing Th2-mediated airway inflammatory responses to HDM ( Fig. 2a ). Bronchoalveolar lavage fluid (BALF) from HDM-challenged WT mice that had received the adoptive transfer of HDM-pulsed BMDCs from WT mice (WT BMDCs) had significant increases in inflammatory cells as compared with HDM-challenged WT mice that had received the adoptive transfer of HDM-pulsed BMDCs from Prkdc scid mice ( scid BMDCs; Fig. 2b ). Similarly, HDM-challenged recipients of adoptively transferred WT BMDCs that had been pulsed with HDM had an increase in peribronchial inflammatory cell infiltrates on lung histology as compared with recipients of HDM-pulsed scid BMDCs ( Fig. 2c ). HDM re-stimulation of cultures of mediastinal lymph node (MLN) cells from HDM-challenged mice showed a significant reduction in the production of the Th2 effector cytokines, interleukin (IL)-4, IL-5 and IL-13, in recipients of scid BMDCs as compared with WT BMDCs ( Fig. 2d ). BALF levels of C–C chemokines that recruit eosinophils and T cells to the lung were also significantly reduced in recipients of scid BMDCs as compared with WT BMDCs ( Fig. 2e–h ). These include CCL24 (eotaxin-2), which interacts with CCR3 to recruit eosinophils, CCL17 (TARC) and CCL22 (MDC), which interacts with CCR4 on Th2 cells, and CCL5 (RANTES), which interacts with CCR5 that is highly expressed on T cells in the lung [25] , [26] . Lastly, serum levels of HDM-specific IgE were significantly reduced in recipients of scid BMDCs as compared with WT BMDCs, thereby demonstrating the reduced ability of scid BMDCs to induce allergic sensitization ( Fig. 2i ). Collectively, these results demonstrate that DNA-PK-deficient DCs are defective in the initiation of HDM-mediated allergic sensitization and Th2-mediated airway inflammatory responses. 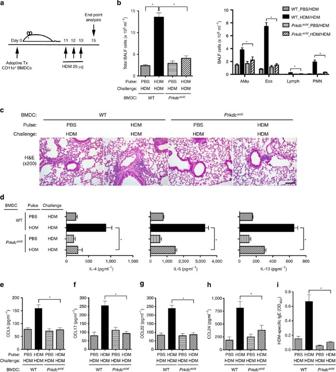Figure 2: The adoptive transfer of HDM-pulsed CD11c+BMDCs fromPrkdcscidmice has a reduced ability to induce allergen-mediated airway inflammation. (a) On day 0, 5 × 104viable CD11c+BMDCs from WT C57BL/6 andPrkdcscidmice, which had been pulsedex vivowith HDM or PBS, as a control, were adoptively transferred to recipient WT C57BL/6 mice. Daily intranasal HDM challenges (25 μg) were administered to all recipient mice on days 11 through 13 and end points were analysed on day 15. (b) Number of total BALF inflammatory cells and inflammatory cell types (alveolar macrophages (AMφ), eosinophils (Eos), lymphocytes (Lymph) and neutrophils (PMN)) from HDM-challenged mice that had received the adoptive transfer of 5 × 104CD11c+BMDCs fromPrkdcscidand WT mice that had been pulsed with either PBS or HDM (n=12–14 mice, *P<0.01, one-way ANOVA with Bonferroni multiple comparison test). (c) Representative histologic lung sections from HDM-challenged mice that had received the adoptive transfer of CD11c+BMDCs fromPrkdcscidand WT mice. Scale bar, 100 μm. (d) Th2 cytokine secretion byex vivocultures of MLN cells that had been re-stimulated with or without HDM (100 μg ml−1;n=3–8 mice, *P<0.05, one-way ANOVA with Bonferroni multiple comparison test). One of two independent experiments that showed similar results is shown (data were not pooled because of different ranges of cytokine production between the two experiments). (e–h) C–C chemokines in BALF (n=11–13 mice, *P<0.01, one-way ANOVA with Bonferroni multiple comparison test). (i) Serum house dust mite-specific IgE (n=8–16 mice, *P<0.0001, one-way ANOVA with Bonferroni multiple comparison test). Results are pooled data from two independent experiments, except where indicated. Figure 2: The adoptive transfer of HDM-pulsed CD11c + BMDCs from Prkdc scid mice has a reduced ability to induce allergen-mediated airway inflammation. ( a ) On day 0, 5 × 10 4 viable CD11c + BMDCs from WT C57BL/6 and Prkdc scid mice, which had been pulsed ex vivo with HDM or PBS, as a control, were adoptively transferred to recipient WT C57BL/6 mice. Daily intranasal HDM challenges (25 μg) were administered to all recipient mice on days 11 through 13 and end points were analysed on day 15. ( b ) Number of total BALF inflammatory cells and inflammatory cell types (alveolar macrophages (AMφ), eosinophils (Eos), lymphocytes (Lymph) and neutrophils (PMN)) from HDM-challenged mice that had received the adoptive transfer of 5 × 10 4 CD11c + BMDCs from Prkdc scid and WT mice that had been pulsed with either PBS or HDM ( n =12–14 mice, * P <0.01, one-way ANOVA with Bonferroni multiple comparison test). ( c ) Representative histologic lung sections from HDM-challenged mice that had received the adoptive transfer of CD11c + BMDCs from Prkdc scid and WT mice. Scale bar, 100 μm. ( d ) Th2 cytokine secretion by ex vivo cultures of MLN cells that had been re-stimulated with or without HDM (100 μg ml −1 ; n =3–8 mice, * P <0.05, one-way ANOVA with Bonferroni multiple comparison test). One of two independent experiments that showed similar results is shown (data were not pooled because of different ranges of cytokine production between the two experiments). ( e – h ) C–C chemokines in BALF ( n =11–13 mice, * P <0.01, one-way ANOVA with Bonferroni multiple comparison test). ( i ) Serum house dust mite-specific IgE ( n =8–16 mice, * P <0.0001, one-way ANOVA with Bonferroni multiple comparison test). Results are pooled data from two independent experiments, except where indicated. Full size image DNA-PK inhibition attenuates Th2 inflammation Experiments were next conducted to assess whether CD11c + BMDCs that had been treated ex vivo with the DNA-PK inhibitor, NU7441, have a reduced ability to induce Th2-mediated allergic airway inflammation in response to HDM ( Fig. 3a ). Recipients of adoptively transferred HDM-pulsed WT DCs that had been treated with NU7441 had significant reductions in the number of BALF inflammatory cells as compared with recipients of HDM-pulsed WT DCs that had been treated with medium alone ( Fig. 3b ). Consistent with this, lung histology showed a reduction in peribronchial inflammatory cell infiltrates in recipients of HDM-pulsed WT DCs that had been treated with NU7441, which was associated with a reduction in mucous cell metaplasia ( Fig. 3c,d ). HDM re-stimulation of ex vivo cultures of MLN cells from recipients of NU7441-treated HDM-pulsed BMDCs had a reduced ability to produce the Th2 cytokines, IL-4, IL-5 and IL-13 as compared with recipients of HDM-pulsed WT DCs treated with the medium alone ( Fig. 3e ). BALF levels of the anti-inflammatory cytokine, IL-10, were significantly higher in recipients of NU7441-treated HDM-pulsed WT DCs ( Fig. 3f ), whereas BALF levels of chemokines (CCL5, CCL17, CCL22 and CCL24) were significantly reduced ( Fig. 3g ). Lastly, serum levels of HDM-specific IgE were significantly reduced in recipients of NU7441-treated HDM-pulsed WT DCs, indicating impaired allergic sensitization ( Fig. 3h ). These results demonstrate that NU7441-mediated pharmacological inhibition of DNA-PK in BMDCs impairs their ability to initiate HDM-mediated allergic sensitization and Th2-mediated airway inflammatory responses. 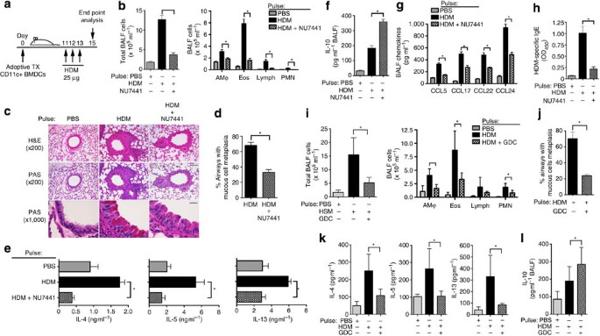Figure 3: The adoptive transfer of HDM-pulsed CD11c+BMDCs treated with the DNA-PK inhibitor, NU7441, or the Akt inhibitor, GDC0068, have an impaired ability to induce allergen-mediated airway inflammation. (a) On day 0, 5 × 104viable CD11c+BMDCs from WT C57BL/6 mice that were pulsedex vivowith HDM (100 μg ml−1) or PBS, with or without 0.5 μM NU7441 (a–h) or 1 μM GDC0068 (i–l), were adoptively transferred to recipient WT mice. Daily intranasal HDM challenges (25 μg) were administered to all recipient mice on days 11 through 13 and end points were analysed on day 15. (b) Number of total BALF cells and inflammatory cell types (alveolar macrophages (AMφ), eosinophils (Eos), lymphocytes (Lymph) and neutrophils (PMN)) from HDM-challenged mice that had received the adoptive transfer of CD11c+BMDCs treated with NU7441 and pulsed with either PBS or HDM (n=12 mice, *P<0.01, one-way ANOVA with Bonferroni multiple comparison test). (c) Representative histologic lung sections stained with haematoxylin and eosin (H&E) or PAS. Scale bars, 100 μm for the × 200 images and 20 μm for the × 1,000 images. (d) Quantification of mucous cell metaplasia (n=12 mice, *P<0.0001, HDM+NU7441 versus HDM alone, Mann–Whitney test). Overall, 54±3 airways were examined per mouse. (e) Th2 cytokine secretion byex vivocultures of MLN cells that had been re-stimulated with PBS or HDM (100 μg ml−1;n=9–16 mice, *P<0.01, HDM versus HDM+NU7441, one-way ANOVA with Bonferroni multiple comparison test). (f) BALF IL-10 (n=12 mice, *P<0.0001, HDM versus HDM+NU7441, one-way ANOVA with Bonferroni multiple comparison test). (g) BALF C–C chemokines (n=12 mice, *P<0.0001, HDM versus HDM+NU7441, one-way ANOVA with Bonferroni multiple comparison test). (h) Serum HDM-specific IgE (n=8–15 mice, *P<0.001, HDM versus HDM+NU7441, one-way ANOVA with Bonferroni multiple comparison test). (i) Number of BALF inflammatory cells from HDM-challenged mice that received the adoptive transfer of CD11c+BMDCs treated with the Akt inhibitor, GDC0068 (GDC), and pulsed with either PBS or HDM (n=8–9 mice, *P<0.001, one-way ANOVA with Sidak’s multiple comparison test). (j) Quantification of mucous cell metaplasia (n=5 mice, *P=0.0079, HDM+GDC0068 (GDC) versus HDM alone, Mann–Whitney test). Overall, 65±2 airways were examined per mouse. (k) Th2 cytokine secretion byex vivocultures of MLN cells that were re-stimulated with PBS or HDM (100 μg ml−1;n=4 mice, *P<0.05, HDM versus HDM+GDC0068, one-way ANOVA with Sidak’s multiple comparison test). Representative results from one of two independent experiments are shown. (l) BALF IL-10 (n=9 mice, *P<0.05, HDM versus HDM+GDC0068, one-way ANOVA with Sidak’s multiple comparison test). Results are pooled data from two independent experiments, unless otherwise indicated. Figure 3: The adoptive transfer of HDM-pulsed CD11c + BMDCs treated with the DNA-PK inhibitor, NU7441, or the Akt inhibitor, GDC0068, have an impaired ability to induce allergen-mediated airway inflammation. ( a ) On day 0, 5 × 10 4 viable CD11c + BMDCs from WT C57BL/6 mice that were pulsed ex vivo with HDM (100 μg ml −1 ) or PBS, with or without 0.5 μM NU7441 ( a – h ) or 1 μM GDC0068 ( i – l ), were adoptively transferred to recipient WT mice. Daily intranasal HDM challenges (25 μg) were administered to all recipient mice on days 11 through 13 and end points were analysed on day 15. ( b ) Number of total BALF cells and inflammatory cell types (alveolar macrophages (AMφ), eosinophils (Eos), lymphocytes (Lymph) and neutrophils (PMN)) from HDM-challenged mice that had received the adoptive transfer of CD11c + BMDCs treated with NU7441 and pulsed with either PBS or HDM ( n =12 mice, * P <0.01, one-way ANOVA with Bonferroni multiple comparison test). ( c ) Representative histologic lung sections stained with haematoxylin and eosin (H&E) or PAS. Scale bars, 100 μm for the × 200 images and 20 μm for the × 1,000 images. ( d ) Quantification of mucous cell metaplasia ( n =12 mice, * P <0.0001, HDM+NU7441 versus HDM alone, Mann–Whitney test). Overall, 54±3 airways were examined per mouse. ( e ) Th2 cytokine secretion by ex vivo cultures of MLN cells that had been re-stimulated with PBS or HDM (100 μg ml −1 ; n =9–16 mice, * P <0.01, HDM versus HDM+NU7441, one-way ANOVA with Bonferroni multiple comparison test). ( f ) BALF IL-10 ( n =12 mice, * P <0.0001, HDM versus HDM+NU7441, one-way ANOVA with Bonferroni multiple comparison test). ( g ) BALF C–C chemokines ( n =12 mice, * P <0.0001, HDM versus HDM+NU7441, one-way ANOVA with Bonferroni multiple comparison test). ( h ) Serum HDM-specific IgE ( n =8–15 mice, * P <0.001, HDM versus HDM+NU7441, one-way ANOVA with Bonferroni multiple comparison test). ( i ) Number of BALF inflammatory cells from HDM-challenged mice that received the adoptive transfer of CD11c + BMDCs treated with the Akt inhibitor, GDC0068 (GDC), and pulsed with either PBS or HDM ( n =8–9 mice, * P <0.001, one-way ANOVA with Sidak’s multiple comparison test). ( j ) Quantification of mucous cell metaplasia ( n =5 mice, * P =0.0079, HDM+GDC0068 (GDC) versus HDM alone, Mann–Whitney test). Overall, 65±2 airways were examined per mouse. ( k ) Th2 cytokine secretion by ex vivo cultures of MLN cells that were re-stimulated with PBS or HDM (100 μg ml −1 ; n =4 mice, * P <0.05, HDM versus HDM+GDC0068, one-way ANOVA with Sidak’s multiple comparison test). Representative results from one of two independent experiments are shown. ( l ) BALF IL-10 ( n =9 mice, * P <0.05, HDM versus HDM+GDC0068, one-way ANOVA with Sidak’s multiple comparison test). Results are pooled data from two independent experiments, unless otherwise indicated. Full size image If Akt is downstream of DNA-PK signalling in DCs, then treatment of adoptively transferred DCs with GDC0068, a pharmacological inhibitor of Akt kinase activity, would be predicted to have the same effect as treatment of BMDCs with NU7441 before adoptive transfer. Consistent with this concept, WT recipient mice that received the adoptive transfer of HDM-pulsed CD11c + BMDCs that had been treated ex vivo with GDC0068 demonstrated significant reductions in the BALF inflammatory cells ( Fig. 3i ) and mucous cell metaplasia ( Fig. 3j ). In addition, recipients of GDC0068-treated HDM-pulsed WT DCs had reductions in Th2 cytokine production by MLN cells that had been re-stimulated ex vivo with HDM ( Fig. 3k ), as well as an increase in BALF IL-10 levels, as compared with recipients of HDM-pulsed WT DCs that had not been treated with GDC0068 ( Fig. 3l ). Collectively, these results are consistent with the conclusion that Akt is downstream of DNA-PK signalling in DCs. CD11c-specific DNA-PKcs knockouts and Th2 inflammation Next, we considered whether the specific deletion of DNA-PKcs in CD11c + DCs would similarly impair the induction of allergic sensitization and Th2 immune response to HDM. DNA-PKcs fl/fl mice were created with loxP sites flanking exons 82 and 83 of the Prkdc gene ( Fig. 4a ). Exons 82 and 83, along with exon 81, comprise the kinase catalytic domain of DNA-PKcs, and human cells with deletions of these exons have both undetectable kinase activity and DNA-PKcs protein expression [27] . The insertion of the LoxP sites in the floxed allele of the Prkdc gene was confirmed by Southern blotting of genomic DNA from DNA-PKcs fl/+ mice ( Fig. 4b ). DNA-PKcs fl/fl mice were bred with CD11c -Cre mice to generate homozygous DNA-PKcs fl/fl ; CD11c -Cre mice in which DNA-PKcs expression is specifically deleted in CD11c + DCs, but not in other cells, such as airway epithelial cells ( Fig. 4c ). As shown in Fig. 4d , DNA-PKcs mRNA levels were 15.5-fold higher in splenic DCs isolated from DNA-PKcs fl/fl as compared with those from DNA-PKcs fl/fl ; Cd11c -Cre mice. The deletion of exons 82 and 83 of the Prkdc gene was further confirmed by sequencing of genomic DNA from CD11c + splenic DCs isolated from DNA-PKcs fl/fl ; CD11c-Cre mice ( Supplementary Fig. 1 ). DNA-PKcs fl/fl ; CD11c -Cre mice then received multiple intranasal HDM challenges to assess the effect of the CD11c-specific deletion of DNA-PKcs on HDM-induced airway inflammation and Th2 responses ( Fig. 5a ). As shown in Fig. 5b , the number of BALF inflammatory cells recovered from HDM-challenged DNA-PKcs fl/fl ; Cd11c -Cre mice were significantly reduced as compared with those from HDM-challenged DNA-PKcs fl/fl mice. Similarly, lung histopathology showed a reduction in the extent of peribronchial inflammatory cell infiltrates in HDM-challenged DNA-PKcs fl/fl ; Cd11c -Cre mice as compared with HDM-challenged DNA-PKcs fl/fl mice ( Fig. 5c ). Mucous cell metaplasia was also significantly reduced in HDM-challenged DNA-PKcs fl/fl ; Cd11c -Cre mice as compared with HDM-challenged DNA-PKcs fl/fl mice ( Fig. 5c,d ). HDM re-stimulation of MLNs from DNA-PKcs fl/fl ; Cd11c -Cre mice showed significant reductions in the Th2 cytokines, IL-5 and IL-13, whereas the reduction in IL-4 production was not statistically significant ( Fig. 5e ). There was also no change in interferon (IFN)-γ production by MLN cells following HDM re-stimulation. BALF levels of C–C chemokines, CCL17, CCL22 and CCL24, were also significantly reduced in HDM-challenged DNA-PKcs fl/fl ; Cd11c -Cre mice as compared with HDM-challenged DNA-PKcs fl/fl mice, whereas there was no difference in levels of CCL5 ( Fig. 5f ). Lastly, there was a significant reduction in serum levels of HDM-specific IgE in HDM-challenged DNA-PKcs fl/fl ; Cd11c -Cre mice ( Fig. 5g ). Collectively, these results demonstrate that DNA-PKcs fl/fl ; Cd11c -Cre mice have an impaired ability to induce both allergic sensitization to HDM and Th2-mediated airway inflammatory responses. 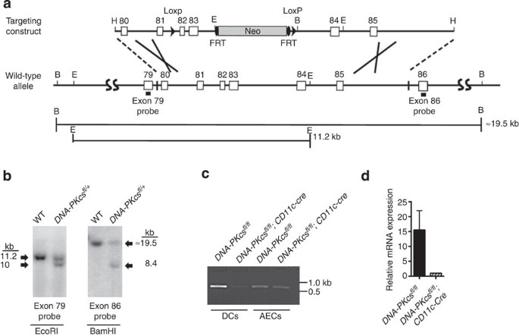Figure 4: Generation and characterization ofDNA-PKcsfl/fl; CD11c-Cremice. (a) TheDNA-PKcsfl/fltargeting construct, consisting of a HindIII fragment containing exons 80–85 of the mousePrkdc gene, is shown at the top, while the WT allele is shown below for comparison. LoxP is shown as an arrowhead, Neo is shown as a cylinder and FRT is shown as an oval. Restriction sites located at the ends of the construct or used in Southern blotting are indicated (H, HindIII; B, BamHI; E, EcoRI). The exon 79 and exon 86 probes used in Southern blotting are shown by solid rectangles. The sizes of the fragments following digestion of the nativePrkdcgene with BamHI or EcoRI are indicated. (b) Southern blots of genomic DNA from WT andDNA-PKcsfl/+mice. Left panel, digestion with EcoRI and detection with an exon 79 probe. Right panel, digestion with BamHI and detection with an exon 86 probe. (c) Genomic DNA from CD11c+/MHCII+/SiglecF−splenic dendritic cells and CD11c−/CD45−/EpcAM+alveolar type II cells isolated from the lungs ofDNA-PKcsfl/flandDNA-PKcsfl/fl; CD11c-Cre mice with flow cytometry. PCR was performed using exon 81 (PKEx81f) and exon 82 (PKEx82r) primers that flank the 5′ loxP site to generate a 646-bp product from the floxed allele, but not from the recombined allele. (SeeSupplementary Figs 3and4for full original images ofb,c.) (d) CD11c+/MHCII+/SiglecF−splenic dendritic cells fromDNA-PKcsfl/flandDNA-PKcsfl/fl; CD11c-Cre mice were sorted using flow cytometry. qRT–PCR was performed on pre-amplified cDNA using a Taqman assay that spanned the junction between exons 82 and 83 ofDNA-PKcsmRNA (each sample represents pooled cells from five mice). Figure 4: Generation and characterization of DNA-PKcs fl/fl ; CD11c-Cre mice. ( a ) The DNA-PKcs fl/fl targeting construct, consisting of a HindIII fragment containing exons 80–85 of the mouse Prkdc gene , is shown at the top, while the WT allele is shown below for comparison. LoxP is shown as an arrowhead, Neo is shown as a cylinder and FRT is shown as an oval. Restriction sites located at the ends of the construct or used in Southern blotting are indicated (H, HindIII; B, BamHI; E, EcoRI). The exon 79 and exon 86 probes used in Southern blotting are shown by solid rectangles. The sizes of the fragments following digestion of the native Prkdc gene with BamHI or EcoRI are indicated. ( b ) Southern blots of genomic DNA from WT and DNA-PKcs fl/+ mice. Left panel, digestion with EcoRI and detection with an exon 79 probe. Right panel, digestion with BamHI and detection with an exon 86 probe. ( c ) Genomic DNA from CD11c + /MHCII + /SiglecF − splenic dendritic cells and CD11c − /CD45 − /EpcAM + alveolar type II cells isolated from the lungs of DNA-PKcs fl/fl and DNA-PKcs fl/fl ; CD11c -Cre mice with flow cytometry. PCR was performed using exon 81 (PKEx81f) and exon 82 (PKEx82r) primers that flank the 5′ loxP site to generate a 646-bp product from the floxed allele, but not from the recombined allele. (See Supplementary Figs 3 and 4 for full original images of b , c .) ( d ) CD11c + /MHCII + /SiglecF − splenic dendritic cells from DNA-PKcs fl/fl and DNA-PKcs fl/fl ; CD11c -Cre mice were sorted using flow cytometry. qRT–PCR was performed on pre-amplified cDNA using a Taqman assay that spanned the junction between exons 82 and 83 of DNA-PKcs mRNA (each sample represents pooled cells from five mice). 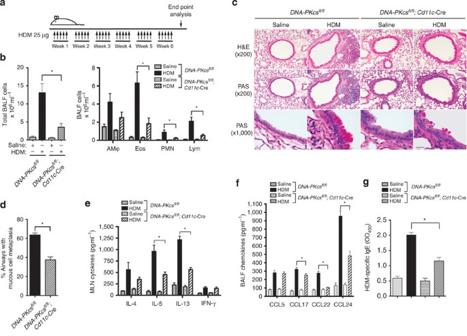Figure 5: HDM-challenged CD11c-specificDNA-PKcsknockout mice have impaired allergen-mediated inflammation. (a)DNA-PKcsfl/flandDNA-PKcsfl/fl; CD11c-Cremice were sensitized and challenged by daily administration of HDM (25 μg) or PBS, 5 days a week, for 6 weeks. End point analysis was performed 72 h after the last administration of HDM. (b) The number of total BALF inflammatory cells and inflammatory cell types (alveolar macrophages (AMφ), eosinophils (Eos), lymphocytes (Lymph) and neutrophils (PMN)) from saline- and HDM-challengedDNA-PKcsfl/fl; CD11c-Cremice were compared withDNA-PKcsfl/flmice, which served as a control (n=8–15 mice, *P<0.01,DNA-PKcsfl/fl; CD11c-cre+HDM versusDNA-PKcsfl/fl+HDM, one-way ANOVA with Bonferroni multiple comparison test). (c) Representative histologic lung sections stained with H&E or PAS are shown. Scale bars, 100 μm for the × 200 images and 20 μm for the × 1,000 images. (d) Quantification of mucous cell metaplasia (n=9 mice, *P<0.0001,DNA-PKcsfl/fl; CD11c-cre+HDM versusDNA-PKcsfl/fl+HDM, unpairedt-test). Overall, 55±3.8 airways were analysed per mouse. (e) Cytokine secretion byex vivocultures of MLN cells that had been re-stimulated with saline or HDM (100 μg ml−1;n=7–13 mice, *P<0.001DNA-PKcsfl/fl; CD11c-cre+HDM versusDNA-PKcsfl/fl+HDM, one-way ANOVA with Bonferroni multiple comparison test). (f) BALF chemokines (n=8–12 mice, *P<0.01,CD11c-cre+HDM versusDNA-PKcsfl/fl+HDM, one-way ANOVA with Bonferroni multiple comparison test). (g) Serum HDM-specific IgE (n=8–16 mice, *P<0.0001,CD11c-cre+HDM versusDNA-PKcsfl/fl+HDM, one-way ANOVA with Bonferroni multiple comparison test). Results are pooled data from two independent experiments. Full size image Figure 5: HDM-challenged CD11c-specific DNA-PKcs knockout mice have impaired allergen-mediated inflammation. ( a ) DNA-PKcs fl/fl and DNA-PKcs fl/fl ; CD11c-Cre mice were sensitized and challenged by daily administration of HDM (25 μg) or PBS, 5 days a week, for 6 weeks. End point analysis was performed 72 h after the last administration of HDM. ( b ) The number of total BALF inflammatory cells and inflammatory cell types (alveolar macrophages (AMφ), eosinophils (Eos), lymphocytes (Lymph) and neutrophils (PMN)) from saline- and HDM-challenged DNA-PKcs fl/fl ; CD11c-Cre mice were compared with DNA-PKcs fl/fl mice, which served as a control ( n =8–15 mice, * P <0.01, DNA-PKcs fl/fl ; CD11c-cre +HDM versus DNA-PKcs fl/fl +HDM, one-way ANOVA with Bonferroni multiple comparison test). ( c ) Representative histologic lung sections stained with H&E or PAS are shown. Scale bars, 100 μm for the × 200 images and 20 μm for the × 1,000 images. ( d ) Quantification of mucous cell metaplasia ( n =9 mice, * P <0.0001, DNA-PKcs fl/fl ; CD11c-cre +HDM versus DNA-PKcs fl/fl +HDM, unpaired t -test). Overall, 55±3.8 airways were analysed per mouse. ( e ) Cytokine secretion by ex vivo cultures of MLN cells that had been re-stimulated with saline or HDM (100 μg ml −1 ; n =7–13 mice, * P <0.001 DNA-PKcs fl/fl ; CD11c-cre +HDM versus DNA-PKcs fl/fl +HDM, one-way ANOVA with Bonferroni multiple comparison test). ( f ) BALF chemokines ( n =8–12 mice, * P <0.01, CD11c-cre +HDM versus DNA-PKcs fl/fl +HDM, one-way ANOVA with Bonferroni multiple comparison test). ( g ) Serum HDM-specific IgE ( n =8–16 mice, * P <0.0001, CD11c-cre +HDM versus DNA-PKcs fl/fl +HDM, one-way ANOVA with Bonferroni multiple comparison test). Results are pooled data from two independent experiments. Full size image Experiments were next conducted to assess the mechanisms by which DNA-PK-deficient CD11c + DCs have a reduced capability to induce allergic sensitization and Th2 immunity to HDM. First, we assessed whether the percentage of T and B cells in naive DNA-PKcs fl/fl and DNA-PKcs fl/fl ; Cd11c -Cre mice were reduced as compared with the WT parental strain of C57BL/6 mice, which could be indicative of a defect in V(D)J recombination with resultant altered lymphocyte development. As shown in Fig. 6a,b , the percentage of CD3 + T cells and CD19 + B cells were not significantly different in the lungs and spleens of naive WT, DNA-PKcs fl/fl and DNA-PKcs fl/fl ; Cd11c -Cre mice, except for an increase in the percentage of splenic CD19 + B cells in DNA-PKcs fl/fl ; Cd11c -Cre mice as compared with WT mice. This finding suggests that lymphocyte development was not significantly impaired in DNA-PKcs fl/fl and DNA-PKcs fl/fl ; Cd11c -Cre mice. Second, we found that cell surface expression of the co-stimulatory molecule, CD80, was significantly reduced on CD11c + DCs in the lungs ( Fig. 6c ) and MLNs ( Fig. 6d ) of HDM-challenged DNA-PKcs fl/fl ; Cd11c -Cre mice as compared with HDM-challenged DNA-PKcs fl/fl mice. Although there were statistically significant differences in the expression of OX-40L, CD40 and CD86 by CD11c + DCs in the lung and MLNs, these differences appeared modest as compared with the reduction in cell surface expression of CD80. In addition, as compared with the murine BMDCs and human moDCs that were utilized for the experiments in Fig. 1h , CD11c + DCs from the lungs and MLNs of DNA-PKcs fl/fl and DNA-PKcs fl/fl ; Cd11c -Cre mice had a different pattern of expression of CD40, CD80 and CD86, as well as lower cell surface levels of these co-stimulatory molecules. 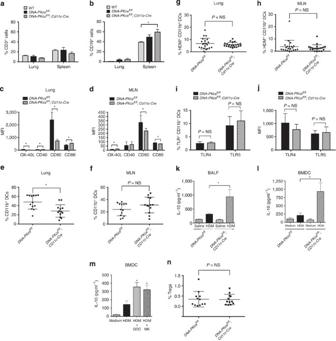Figure 6: Characterization of HDM-challenged CD11c-specificDNA-PKcsknockout mice. (a,b) The percentage of CD3+T cells (a) and CD19+B cells (b) in lungs and spleens of naive, WT C57BL/6 mice, which is the parental strain of bothDNA-PKcsfl/flmice andDNA-PKcsfl/fl; CD11c-Cremice (n=6, *P<0.05, one-way ANOVA with Sidak’s multiple comparison test). Pooled data from two independent experiments. (c,d) MFI of OX-40L, CD40, CD80 and CD86 expression by CD11c+/MHCIIhi/SSCloDCs in lungs (c) and MLN (d) of HDM-challengedDNA-PKcsfl/flmice andDNA-PKcsfl/fl; CD11c-Cremice (n=5–6 mice, *P<0.05, Mann–Whitney test). (e,f) The percentage of CD11c+/MHCIIhi/SSCloDCs that express CD11b in the lungs (e) and MLNs (f) of HDM-challengedDNA-PKcsfl/flmice andDNA-PKcsfl/fl; CD11c-Cremice (n=13 mice, *P<0.0025, Mann–Whitney test). (g,h) Uptake of HDM by CD11c+/MHCIIhi/SSClo/CD11b+DCs in the lungs (g) and MLNs (h) ofDNA-PKcsfl/flmice andDNA-PKcsfl/fl; CD11c-Cremice 72 h after the administration of HDM extract (50 μg) labelled with Alexa Fluor 647 (n=21 mice,P=NS, unpairedt-test). (i,j) The percentage of CD11c+/MHCIIhi/SSClo/CD11b+DCs that express TLR4 or TLR5 (i) and the MFI of TLR4 and TLR5 expression (j) by CD11c+/MHCIIhi/SSClo/CD11b+DCs in the lungs ofDNA-PKcsfl/flmice andDNA-PKcsfl/fl; CD11c-Cremice (n=8 mice,P=NS, Mann–Whitney test). (k) BALF IL-10 (n=9, *P<0.01,DNA-PKcsfl/fl; CD11c-Cre+HDM versusDNA-PKcsfl/fl+HDM, one-way ANOVA with Bonferroni multiple comparison test). (l) IL-10 secretion by BMDCs (n=7–9, *P<0.01,DNA-PKcsfl/fl; CD11c-Cre+HDM versusDNA-PKcsfl/fl+HDM, one-way ANOVA with Bonferroni multiple comparison test). (m) IL-10 secretion by BMDCs stimulated with HDM (100 μg ml−1) with or without Akt inhibitors, GDC0068 (GDC) and MK2206 (MK), both at 1 μM for 24 h (n=8, *P<0.05, HDM versus HDM+Akt inhibitor, one-way ANOVA with Bonferroni multiple comparison test). Pooled data from two independent experiments. (n) The percentage of CD3+/CD4+/CD25+/Foxp3+Tregs in MLNs from saline- and HDM-challengedDNA-PKcsfl/fl; CD11c-Cre mice were compared withDNA-PKcsfl/flmice, which served as a control (n=12 mice,P=NS, Mann–Whitney test). Figure 6: Characterization of HDM-challenged CD11c-specific DNA-PKcs knockout mice. ( a , b ) The percentage of CD3 + T cells ( a ) and CD19 + B cells ( b ) in lungs and spleens of naive, WT C57BL/6 mice, which is the parental strain of both DNA-PKcs fl/fl mice and DNA-PKcs fl/fl ; CD11c-Cre mice ( n =6, * P <0.05, one-way ANOVA with Sidak’s multiple comparison test). Pooled data from two independent experiments. ( c , d ) MFI of OX-40L, CD40, CD80 and CD86 expression by CD11c + /MHCII hi /SSC lo DCs in lungs ( c ) and MLN ( d ) of HDM-challenged DNA-PKcs fl/fl mice and DNA-PKcs fl/fl ; CD11c-Cre mice ( n =5–6 mice, * P <0.05, Mann–Whitney test). ( e , f ) The percentage of CD11c + /MHCII hi /SSC lo DCs that express CD11b in the lungs ( e ) and MLNs ( f ) of HDM-challenged DNA-PKcs fl/fl mice and DNA-PKcs fl/fl ; CD11c-Cre mice ( n =13 mice, * P <0.0025, Mann–Whitney test). ( g , h ) Uptake of HDM by CD11c + /MHCII hi /SSC lo /CD11b + DCs in the lungs ( g ) and MLNs ( h ) of DNA-PKcs fl/fl mice and DNA-PKcs fl/fl ; CD11c-Cre mice 72 h after the administration of HDM extract (50 μg) labelled with Alexa Fluor 647 ( n =21 mice, P =NS, unpaired t -test). ( i , j ) The percentage of CD11c + /MHCII hi /SSC lo /CD11b + DCs that express TLR4 or TLR5 ( i ) and the MFI of TLR4 and TLR5 expression ( j ) by CD11c + /MHCII hi /SSC lo /CD11b + DCs in the lungs of DNA-PKcs fl/fl mice and DNA-PKcs fl/fl ; CD11c-Cre mice ( n =8 mice, P =NS, Mann–Whitney test). ( k ) BALF IL-10 ( n =9, * P <0.01, DNA-PKcs fl/fl ; CD11c-Cre +HDM versus DNA-PKcs fl/fl +HDM, one-way ANOVA with Bonferroni multiple comparison test). ( l ) IL-10 secretion by BMDCs ( n =7–9, * P <0.01, DNA-PKcs fl/fl ; CD11c-Cre +HDM versus DNA-PKcs fl/fl +HDM, one-way ANOVA with Bonferroni multiple comparison test). ( m ) IL-10 secretion by BMDCs stimulated with HDM (100 μg ml −1 ) with or without Akt inhibitors, GDC0068 (GDC) and MK2206 (MK), both at 1 μM for 24 h ( n =8, * P <0.05, HDM versus HDM+Akt inhibitor, one-way ANOVA with Bonferroni multiple comparison test). Pooled data from two independent experiments. ( n ) The percentage of CD3 + /CD4 + /CD25 + /Foxp3 + Tregs in MLNs from saline- and HDM-challenged DNA-PKcs fl/fl ; CD11c -Cre mice were compared with DNA-PKcs fl/fl mice, which served as a control ( n =12 mice, P =NS, Mann–Whitney test). Full size image Next, we focused on CD11b + DCs, as these have been shown to be the primary DC subset that mediates antigen presentation and Th2 immunity [28] , [29] , [30] . We show that the percentage of CD11c + DCs that express CD11b was modestly reduced in the lungs ( Fig. 6e ), but not in the MLNs ( Fig. 6f ) of DNA-PKcs fl/fl ; Cd11c -Cre mice as compared with DNA-PKcs fl/fl mice. Next, to assess the functional significance of the reduction in numbers of CD11b + DCs, AF647-labelled HDM was administered to the lungs of DNA-PKcs fl/fl ; Cd11c -Cre and DNA-PKcs fl/fl mice. As shown in Fig. 6g,h , there was no difference in either uptake of HDM antigen in the lung or subsequent migration to MLNs by CD11c + /MHCII + /CD11b + DCs from DNA-PKcs fl/fl ; Cd11c -Cre mice as compared with DNA-PKcs fl/fl mice. Lastly, since DNA-PK has been reported to modulate the expression of toll-like receptors (TLR) in RAW264.7 macrophages by interacting with the autoimmune regulator, Aire, we assessed whether TLR expression by lung CD11b + DCs was modified in DNA-PKcs fl/fl ; Cd11c -Cre mice as a possible mechanism by which T-cell priming might be impaired [31] . As shown in Fig. 6i,j , there was no difference in the percentage of lung CD11b + DCs that expressed TLR4 or TLR5, or the mean fluorescence intensity (MFI) of TLR4 and TLR5 expression by lung CD11b + DCs, in DNA-PKcs fl/fl as compared with DNA-PKcs fl/fl ; Cd11c -Cre mice. Thus, modified expression of TLR4 or TLR5 by lung CD11b + DCs does not appear to mediate impaired T-cell priming to HDM in DNA-PKcs fl/fl ; Cd11c -Cre mice. This is consistent with prior reports, which found that expression of TLR4 by structural cells, such as airway epithelial cells, but not haematopoietic cells, such as DCs, mediates priming of Th2 cells to HDM through the airway, whereas both haematopoietic and structural cells are required for maximal TLR5-mediated allergic sensitization [32] , [33] . We then assessed whether production of the anti-inflammatory cytokine, IL-10, was modified in DNA-PKcs fl/fl ; Cd11c -Cre mice as a mechanism by which HDM-associated inflammatory responses are decreased. As shown in Fig. 6k , IL-10 was higher in BALF from HDM-challenged DNA-PKcs fl/fl ; Cd11c -Cre mice as compared with HDM-challenged DNA-PKcs fl/fl mice. Furthermore, BMDCs from DNA-PKcs fl/fl ; Cd11c -Cre mice secreted larger amounts of IL-10 in response to HDM stimulation as compared with those from DNA-PKcs fl/fl mice ( Fig. 6l ). Lastly, IL-10 secretion by HDM-stimulated BMDCs from DNA-PKcs fl/fl mice was increased in response to GDC0068 and MK2206, pharmacological inhibitors of Akt, which is downstream of DNA-PK signalling ( Fig. 6m ). Collectively, these results suggest that HDM-induced IL-10 production by DCs is suppressed via a DNA-PKcs/Akt pathway. We also assessed whether the number of CD3 + /CD4 + /CD25 + /Foxp3 + regulatory T cells (Tregs) was modified in DNA-PKcs fl/fl ; Cd11c-Cre mice. However, we found that there was no difference in the percentage of Tregs in MLNs of HDM-challenged DNA-PKcs fl/fl ; Cd11c -Cre mice as compared with DNA-PKcs fl/fl mice ( Fig. 6n ). DNA-PK-deficient CD11b + DCs and antigen presentation Since the uptake of HDM antigen in the lung and its trafficking to MLNs by CD11b + DCs from DNA-PKcs fl/fl ; Cd11c -Cre mice were not reduced, we next assessed whether CD11b + DCs from DNA-PKcs fl/fl ; Cd11c -Cre mice have an impairment in antigen presentation that limits their ability to induce allergic sensitization and Th2-mediated airway inflammation. CD11b + DCs were isolated from MLNs of DNA-PKcs fl/fl and DNA-PKcs fl/fl ; Cd11c -Cre mice that had been challenged with HDM or saline and adoptively transferred to WT mice that subsequently received intranasal HDM challenges to induce airway inflammation ( Fig. 7a ). As shown in Fig. 7b , the number of alveolar macrophages, eosinophils, neutrophils and lymphocytes were significantly reduced in BALF from recipients of CD11b + DCs from DNA-PKcs fl/fl ; Cd11c -Cre donor mice as compared with DNA-PKcs fl/fl donor mice. Similarly, lung histology showed a reduction in peribronchial inflammatory cell infiltrates and mucous cell metaplasia in recipients of CD11b + DCs from DNA-PKcs fl/fl ; Cd11c -Cre donor mice as compared with DNA-PKcs fl/fl donor mice ( Fig. 7c,d ). Serum levels of HDM-specific IgE were significantly reduced in recipients of CD11b + DCs from DNA-PKcs fl/fl ; Cd11c -Cre donor mice, while ex vivo cultures of MLNs that had been re-stimulated with HDM showed an impaired ability to produce IL-5 and IL-13 ( Fig. 7e,f ). Collectively, these experiments demonstrate that CD11b + DCs from DNA-PKcs fl/fl ; Cd11c -Cre mice have an impairment in antigen presentation and the subsequent induction of allergic sensitization and Th2 immunity to HDM. 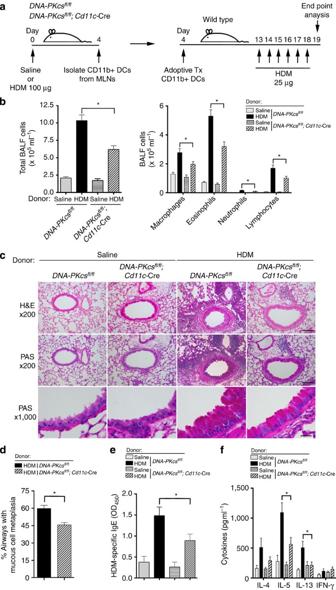Figure 7: The adoptive transfer of CD11b+DCs from Cd11c-specificDNA-PKcsknockout mice has an impaired ability to induce HDM-mediated airway inflammation. (a)DNA-PKcsfl/flandDNA-PKcsfl/fl; CD11c-Credonor mice received a single intranasal dose of 100 μg of HDM extract or saline and after 4 days, MLNs were removed and CD11c+/CD11b+/SiglecF−/MHCII+DCs were isolated with flow cytometry. Overall, 2.5 × 104CD11c+/CD11b+/SiglecF−/MHCII+DCs were adoptively transferred to WT C57BL6 recipient mice by intranasal administration on day 4 and daily intranasal HDM challenges (25 μg) were administered on days 13 through 18 to all recipient mice. Mice were killed for end point analysis on day 19. (b) The number of total BALF inflammatory cells and inflammatory cell subtypes in recipients of adoptively transferred CD11b+DCs (n=6–10, *P<0.05, one-way ANOVA with Bonferroni multiple comparison test). (c) Representative histologic lung sections stained with H&E and PAS. Scale bars, 100 μm for the × 200 images and 20 μm for the × 1,000 images. (d) Quantification of mucous cell metaplasia (n=10, *P=0.0005, unpairedt-test). Overall, 48.7±3.3 airways were analysed per mouse. (e) Serum HDM-specific IgE (n=6–10 mice, *P<0.05, one-way ANOVA with Bonferroni multiple comparison test). (f) Cytokine secretion byex vivocultures of MLN cells that had been re-stimulated with HDM (100 μg ml−1;n=6–8 mice, *P<0.01, one-way ANOVA with Bonferroni multiple comparison test). Results are pooled data from two independent experiments. Figure 7: The adoptive transfer of CD11b + DCs from Cd11c-specific DNA-PKcs knockout mice has an impaired ability to induce HDM-mediated airway inflammation. ( a ) DNA-PKcs fl/fl and DNA-PKcs fl/fl ; CD11c-Cre donor mice received a single intranasal dose of 100 μg of HDM extract or saline and after 4 days, MLNs were removed and CD11c + /CD11b + /SiglecF − /MHCII + DCs were isolated with flow cytometry. Overall, 2.5 × 10 4 CD11c + /CD11b + /SiglecF − /MHCII + DCs were adoptively transferred to WT C57BL6 recipient mice by intranasal administration on day 4 and daily intranasal HDM challenges (25 μg) were administered on days 13 through 18 to all recipient mice. Mice were killed for end point analysis on day 19. ( b ) The number of total BALF inflammatory cells and inflammatory cell subtypes in recipients of adoptively transferred CD11b + DCs ( n =6–10, * P <0.05, one-way ANOVA with Bonferroni multiple comparison test). ( c ) Representative histologic lung sections stained with H&E and PAS. Scale bars, 100 μm for the × 200 images and 20 μm for the × 1,000 images. ( d ) Quantification of mucous cell metaplasia ( n =10, * P =0.0005, unpaired t -test). Overall, 48.7±3.3 airways were analysed per mouse. ( e ) Serum HDM-specific IgE ( n =6–10 mice, * P <0.05, one-way ANOVA with Bonferroni multiple comparison test). ( f ) Cytokine secretion by ex vivo cultures of MLN cells that had been re-stimulated with HDM (100 μg ml −1 ; n =6–8 mice, * P <0.01, one-way ANOVA with Bonferroni multiple comparison test). Results are pooled data from two independent experiments. Full size image Inhibition of DNA-PK suppresses HDM-induced airway disease Lastly, we assessed whether pharmacologic inhibition of DNA-PK by consumption of chow containing NU7441 could attenuate HDM-induced airway disease in WT mice, which could provide evidence to support the concept of utilizing DNA-PK inhibitors for the treatment of asthmatic patients ( Fig. 8a ). As shown in Fig. 8b , mice that consumed chow containing 0.6 or 0.9% NU7441 had similar significant decreases in the number of BALF inflammatory cells. Lung histopathology similarly revealed that mice that were fed NU7441 had reductions in peribronchial inflammatory cell infiltrates ( Fig. 8c ). In addition to the reductions in airway inflammation, NU7441 also attenuated HDM-mediated increases in mucous cell metaplasia ( Fig. 8d ) and airway hyper-responsiveness (AHR; Fig. 8e ). The reductions in airway inflammation and AHR were similar in mice that received chow containing either 0.6 or 0.9% NU7441. 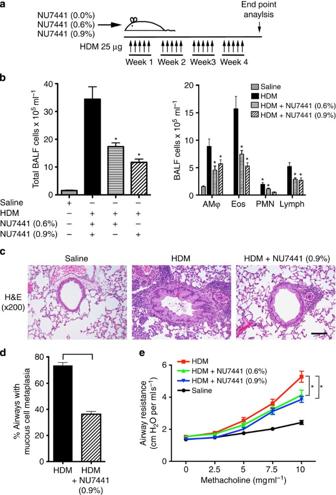Figure 8: Oral administration of the DNA-PK inhibitor, NU7441, attenuates HDM-induced allergic inflammation, mucous cell metaplasia and airway hyper-responsiveness. (a) WT BALB/c mice were sensitized and challenged by daily intranasal administration of HDM (25 μg) or PBS, 5 days a week for 4 weeks. Mice were fed chow that contained 0, 0.6 or 0.9% NU7441 coincident with the HDM sensitization and challenges. (b) The number of total BALF inflammatory cells and inflammatory cell types (alveolar macrophages (AMφ), eosinophils (Eos), neutrophils (PMN) and lymphocytes (Lymph)) from saline- and HDM-challenged BALB/c mice that had or had not been fed chow containing 0.6 or 0.9% NU7441 (n=20–35 mice, *P<0.05, HDM versus HDM+NU7441, one-way ANOVA with Bonferroni multiple comparison test). (c) Representative histologic lung sections stained with H&E. Scale bar, 100 μm. (d) Quantification of mucous cell metaplasia (n=20 mice, *P<0.0001, HDM+NU7441 versus HDM alone, unpairedt-test). Overall, 45±2 airways were examined per mouse. (e) Airway resistance (cm H2O per ml s−1) to inhaled methacholine (n=17–20 mice, *P<0.001, HDM versus HDM+NU7441, two-way ANOVA with Bonferroni post test). Results are pooled data from two independent experiments. Figure 8: Oral administration of the DNA-PK inhibitor, NU7441, attenuates HDM-induced allergic inflammation, mucous cell metaplasia and airway hyper-responsiveness. ( a ) WT BALB/c mice were sensitized and challenged by daily intranasal administration of HDM (25 μg) or PBS, 5 days a week for 4 weeks. Mice were fed chow that contained 0, 0.6 or 0.9% NU7441 coincident with the HDM sensitization and challenges. ( b ) The number of total BALF inflammatory cells and inflammatory cell types (alveolar macrophages (AMφ), eosinophils (Eos), neutrophils (PMN) and lymphocytes (Lymph)) from saline- and HDM-challenged BALB/c mice that had or had not been fed chow containing 0.6 or 0.9% NU7441 ( n =20–35 mice, * P <0.05, HDM versus HDM+NU7441, one-way ANOVA with Bonferroni multiple comparison test). ( c ) Representative histologic lung sections stained with H&E. Scale bar, 100 μm. ( d ) Quantification of mucous cell metaplasia ( n =20 mice, * P <0.0001, HDM+NU7441 versus HDM alone, unpaired t -test). Overall, 45±2 airways were examined per mouse. ( e ) Airway resistance (cm H 2 O per ml s −1 ) to inhaled methacholine ( n =17–20 mice, * P <0.001, HDM versus HDM+NU7441, two-way ANOVA with Bonferroni post test). Results are pooled data from two independent experiments. Full size image Additional experiments were performed to characterize further the effects of NU7441 on indices of airway inflammation. As shown in Fig. 9a , HDM re-stimulation of ex vivo MLN cultures from mice that had been fed chow containing NU7441 showed significant reductions in the production of the Th2 cytokines, IL-5 and IL-13, with or without ex vivo treatment with NU7441. Similarly, the number of BALF CD4 + T cells were reduced in HDM-challenged mice that were fed chow containing NU7441, as were the number of IL-5 + CD4 + T cells, whereas the number of IL-13 + CD4 + T cells appeared to be decreased, but did not reach statistical significance ( Fig. 9b ). The number of IL-17 + CD4 + T cells, however, was not reduced ( Fig. 9b ). Mice that received NU7441 also had an increase in BALF IL-10 levels ( Fig. 9c ) and a reduction in BALF CCL24 ( Fig. 9d ). NU7441 also attenuated allergic sensitization as indicated by reduced plasma levels of HDM-specific IgE ( Fig. 9e ). Collectively, these findings demonstrate that oral administration of a pharmacological DNA-PK inhibitor can attenuate allergen sensitization and Th2-mediated airway inflammation, as well as other cardinal manifestations of experimental HDM-induced asthma, including mucous cell metaplasia and AHR. 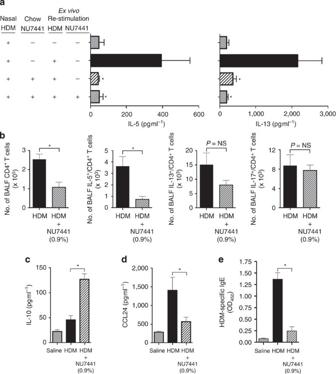Figure 9: Oral administration of the DNA-PK inhibitor, NU7441, attenuates HDM-induced allergic inflammation and IgE production. (a) Th2 cytokine production by MLN cells from HDM-challenged mice that had or had not been fed chow containing 0.9% NU7441 and re-stimulatedex vivowith or without HDM (100 μg ml−1) and NU7441 (0.5 μM;n=6–12 mice, *P<0.05, versus HDM, one-way ANOVA with Bonferroni multiple comparison test). (b) The total number of CD4+T cells, as well as IL-5+/CD4+and IL-13+/CD4+T cells in BALF, was quantified by flow cytometry (n=10 mice, *P<0.01, Mann–Whitney test). (c) BALF IL-10 (n=7–12 mice, *P<0.001, one-way ANOVA with Bonferroni multiple comparison test). (d) BALF CCL24 (n=19–36 mice, *P<0.01, one-way ANOVA with Bonferroni multiple comparison test). (e) Serum HDM-specific IgE (n=16 mice, *P<0.001, one-way ANOVA with Bonferroni multiple comparison test). Results are pooled data from at least two independent experiments. Figure 9: Oral administration of the DNA-PK inhibitor, NU7441, attenuates HDM-induced allergic inflammation and IgE production. ( a ) Th2 cytokine production by MLN cells from HDM-challenged mice that had or had not been fed chow containing 0.9% NU7441 and re-stimulated ex vivo with or without HDM (100 μg ml −1 ) and NU7441 (0.5 μM; n =6–12 mice, * P <0.05, versus HDM, one-way ANOVA with Bonferroni multiple comparison test). ( b ) The total number of CD4 + T cells, as well as IL-5 + /CD4 + and IL-13 + /CD4 + T cells in BALF, was quantified by flow cytometry ( n =10 mice, * P <0.01, Mann–Whitney test). ( c ) BALF IL-10 ( n =7–12 mice, * P <0.001, one-way ANOVA with Bonferroni multiple comparison test). ( d ) BALF CCL24 ( n =19–36 mice, * P <0.01, one-way ANOVA with Bonferroni multiple comparison test). ( e ) Serum HDM-specific IgE ( n =16 mice, * P <0.001, one-way ANOVA with Bonferroni multiple comparison test). Results are pooled data from at least two independent experiments. Full size image Lastly, experiments were performed to assess the effect of treatment with NU7441 after T-cell priming had already occurred. As shown in Fig. 10a , HDM-sensitized WT mice that consumed chow containing 0.9% NU7441 concurrent with intranasal HDM challenges, but after allergic sensitization had already occurred, demonstrated a significant reduction in the number of BALF inflammatory cells ( Fig. 10b,c ), as well as in the extent of peribronchial inflammation on lung histology ( Fig. 10d ). NU7441 (0.9%) treatment was also associated with reductions in serum levels of HDM-specific IgE ( Fig. 10e ), mucous cell metaplasia ( Fig. 10d,f ) and AHR ( Fig. 10g ), whereas BALF IL-10 levels were significantly increased ( Fig. 10h ). This demonstrates that oral administration of a pharmacological DNA-PK inhibitor only during the challenge phase can similarly attenuate the manifestations of HDM-induced asthma. 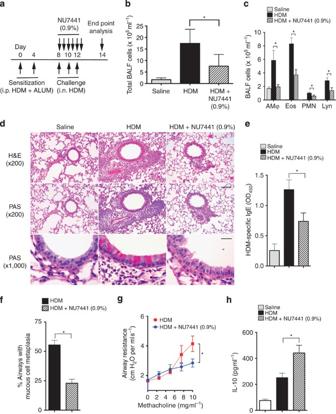Figure 10: Oral administration of the DNA-PK inhibitor, NU7441, during the challenge phase attenuates the manifestations of experimental HDM-induced asthma. (a) WT BALB/c mice were sensitized by intraperitoneal administration of HDM (100 μg) and aluminium hydroxide (3 mg) on days 0 and 4. Mice received intranasal challenges with HDM (100 μg) on days 8, 10 and 12 to induce experimental asthma and were concurrently fed chow that contained NU7441 (0.9%) on days 8 through 12. End points were assessed on day 14. (b,c) The number of total BALF inflammatory cells (b) and inflammatory cell types (alveolar macrophages (AMφ), eosinophils (Eos), neutrophils (PMN) and lymphocytes (Lymph)) (c) were significantly reduced in HDM-challenged WT mice that had been fed chow containing NU7441 (0.9%) during the challenge phase as compared with WT mice that had received regular chow (n=10 mice, *P<0.05, HDM versus HDM+NU7441 (0.9%), one-way ANOVA with Sidak’s multiple comparison test). (d) Representative histologic lung sections stained with H&E. Scale bars, 100 μm for the × 200 images and 20 μm for the × 1,000 images. (e) Serum levels of HDM-specific IgE were quantified by ELISA (n=10 mice, *P<0.05, HDM versus HDM+NU7441 (0.9%), one-way ANOVA with Sidak’s multiple comparison test). (f) Quantification of mucous cell metaplasia (n=10 mice, *P<0.0001, HDM versus HDM+NU7441 (0.9%), unpairedt-test). Overall, 58.4±2.8 airways were examined per mouse. (g) Airway resistance (cm H2O per ml s−1) to inhaled methacholine (10 mg ml−1) was significantly reduced in mice that were fed chow that contained NU7441 (0.9%;n=10 mice, *P=, HDM versus HDM+NU7441, unpairedt-test). (h) BALF IL-10 (n=10 mice, *P<0.01, HDM versus HDM+NU7441 (0.9%), one-way ANOVA with Sidak’s multiple comparison test). Figure 10: Oral administration of the DNA-PK inhibitor, NU7441, during the challenge phase attenuates the manifestations of experimental HDM-induced asthma. ( a ) WT BALB/c mice were sensitized by intraperitoneal administration of HDM (100 μg) and aluminium hydroxide (3 mg) on days 0 and 4. Mice received intranasal challenges with HDM (100 μg) on days 8, 10 and 12 to induce experimental asthma and were concurrently fed chow that contained NU7441 (0.9%) on days 8 through 12. End points were assessed on day 14. ( b , c ) The number of total BALF inflammatory cells ( b ) and inflammatory cell types (alveolar macrophages (AMφ), eosinophils (Eos), neutrophils (PMN) and lymphocytes (Lymph)) ( c ) were significantly reduced in HDM-challenged WT mice that had been fed chow containing NU7441 (0.9%) during the challenge phase as compared with WT mice that had received regular chow ( n =10 mice, * P <0.05, HDM versus HDM+NU7441 (0.9%), one-way ANOVA with Sidak’s multiple comparison test). ( d ) Representative histologic lung sections stained with H&E. Scale bars, 100 μm for the × 200 images and 20 μm for the × 1,000 images. ( e ) Serum levels of HDM-specific IgE were quantified by ELISA ( n =10 mice, * P <0.05, HDM versus HDM+NU7441 (0.9%), one-way ANOVA with Sidak’s multiple comparison test). ( f ) Quantification of mucous cell metaplasia ( n =10 mice, * P <0.0001, HDM versus HDM+NU7441 (0.9%), unpaired t -test). Overall, 58.4±2.8 airways were examined per mouse. ( g ) Airway resistance (cm H 2 O per ml s −1 ) to inhaled methacholine (10 mg ml −1 ) was significantly reduced in mice that were fed chow that contained NU7441 (0.9%; n =10 mice, * P =, HDM versus HDM+NU7441, unpaired t -test). ( h ) BALF IL-10 ( n =10 mice, * P <0.01, HDM versus HDM+NU7441 (0.9%), one-way ANOVA with Sidak’s multiple comparison test). Full size image DCs are the primary antigen-presenting cells in the lung that induce allergic sensitization and Th2 adaptive immune responses to inhaled allergens, such as HDM, which is a common aeroallergen that causes asthma [34] , [35] . DCs that reside in the airway take up antigens for processing in the context of MHCII, followed by migration to MLNs where they facilitate Th2 cell differentiation and production of the key effector cytokines, such as IL-5 and IL-13. Consistent with this, transgenic mice that have been depleted of CD11c + DCs are not capable of mounting Th2 responses to HDM or HDM-induced pulmonary eosinophilia and lymphocytosis, whereas the adoptive transfer of CD11c + /MHCII + cells is sufficient to induce Th2 immunity and pulmonary eosinophilia and lymphocytosis [35] . Limited and conflicting data, however, exist regarding the role of DNA-PK in DC function [36] , [37] , [38] . Prior studies using splenic CD11c + DCs and BMDCs from DNA-PKcs −/− mice have found that DNA-PK was not required for production of IFN-α and IL-12 in response to oligodeoxynucleotides that contained unmethylated CpG motifs (CpG-ODN), which instead signalled via TLR9 and MyD88 (refs 36 , 37 ). A recent publication, however, has shown that BMDCs from DNA-PKcs −/− mice had reduced CpG-ODN-mediated production of IL-6 and IL-12 (ref. 38 ). Furthermore, CpG-ODN was shown to bind DNA-PKcs and induce its association with TRAF6. Here we investigated whether DNA-PK participated in DC-mediated induction of allergic sensitization to HDM and Th2-mediated airway inflammation. First, we show that DNA-PK is phosphorylated and activated in DCs in response to HDM stimulation by a mechanism that is dependent upon the generation of intracellular ROS. This is consistent with prior reports demonstrating that factors that activate DNA-PK are not restricted to DSB, but also include ROS and hypoxia [39] , [40] , [41] . We also show that the DNA-PK inhibitor, NU7441, as well as ROS inhibitors, NAC and DPI, attenuate HDM-mediated phosphorylation of Akt on Ser 473 and Thr 308 . This is consistent with the ability of DNA-PK to function as an upstream kinase that associates with and phosphorylates Akt on Ser 473 , especially in the setting of DSB [42] , [43] . This is also highly relevant to the induction of HDM-mediated allergic immune responses, as Akt signalling has been reported to regulate the activation and antigen-presenting capability of DCs [23] . We also showed that HDM-stimulated BMDCs from Prkdc scid mice were defective in ROS generation. DCs endogenously generate ROS during antigen presentation and ROS functions as a second messenger for MHCII-restricted antigen presentation with resultant activation of CD4 + Th2 cells to produce effector cytokines [44] , [45] , [46] , [47] , [48] . Therefore, we hypothesized that in the absence of DNA-PK, DCs might have an impaired ability to induce Th2-mediated adaptive immune responses to HDM. Here we utilized several experimental models to demonstrate a key role for DNA-PK in the induction of allergic sensitization and Th2 effector cytokine production by DCs in response to HDM. First, we showed that the adoptive transfer of HDM-pulsed CD11c + BMDCs from Prkdc scid mice or WT CD11c + BMDCs that had been treated with the DNA-PK inhibitor, NU7441, had an impaired ability to induce allergic sensitization, as indicated by a decrease in serum levels of HDM-specific IgE, as well as a reduction in production of Th2 effector cytokines, C–C chemokines and HDM-mediated airway inflammation. Next, a CD11c-conditional DNA-PKcs-deficient mouse was created to characterize further the role of DNA-PK expression by DCs in allergic sensitization. Similar to the adoptive transfer experiments, HDM-challenged DNA-PKcs fl/fl ; CD11c-Cre mice displayed a phenotype of impaired allergic sensitization and attenuated induction of Th2 immune responses to HDM that were associated with reductions in C–C chemokine production, airway inflammation and mucous cell metaplasia. Furthermore, CD11c + DCs in the lungs and MLNs from HDM-challenged DNA-PKcs fl/fl ; CD11c-Cre mice had reduced cell surface expression of the co-stimulatory molecule, CD80, which mediates signal 2 signalling via binding CD28 on T cells [49] . CD11b + DCs have been shown to be specialized for antigen presentation in the context of MHCII and induce Th2 responses via the expression of IRF4 (interferon regulatory factor-4) target genes, whereas CD11b − DCs, whose main function is to mediate MHCI-restricted cytotoxic T-lymphocyte responses via the expression of IFN regulatory factor-8 and basic leucine zipper transcription factor (ATF-like 3) can prime MHCII-restricted T-cell responses only at high doses of antigen [30] . Consistent with this, CD11b + DCs play an important role in mediating Th2 effector responses to HDM [28] , [29] . CD11b + conventional DCs have been identified as the key DC subset that mediates the presentation of HDM antigens and the induction of Th2-mediated eosinophilic airway inflammation, whereas the primary role of CD11b + moDCs is to generate pro-inflammatory cytokines, although they can also induce Th2-mediated immunity to HDM [29] . Here we show that CD11b + DCs that had been isolated from the MLNs of HDM-challenged DNA-PKcs fl/fl ; CD11c Cre mice displayed impaired antigen presentation upon adoptive transfer to WT mice that was associated with attenuated airway inflammation. This also demonstrates that the antigen presentation defect was not a consequence of deletion of DNA-PKcs in other CD11c + cells in the lung, such as alveolar macrophages. Furthermore, we found that neither uptake of HDM antigen nor subsequent migration to MLNs were impaired in CD11b + DCs from DNA-PKcs fl/fl ; CD11c-Cre mice. Collectively, these results demonstrate that DNA-PK-deficient CD11b + DCs have a defect in antigen presentation that results in attenuated allergic sensitization and Th2 immune responses to HDM. IL-10 is an important anti-inflammatory cytokine that attenuates the functions of a variety of cell types that are relevant to the pathogenesis of asthma, including DCs [50] , [51] . In particular, IL-10 suppresses several key DC functions, including antigen presentation, cellular maturation, expression of MHCII and co-stimulatory molecules, production of pro-inflammatory cytokines and activation of Akt and NF-κB signalling pathways [23] , [50] , [52] . Furthermore, mature pulmonary DCs can produce IL-10 in response to OVA challenge and thereby mediate antigen-specific T-cell unresponsiveness indicative of immunologic tolerance, while IL-10 gene delivery to the lung suppresses Th2 inflammation, as well as antigen presentation and migration to MLNs by CD11c + DCs [53] , [54] . Myeloid DCs have also been shown to produce IL-10 via TLR-dependent and TLR-independent pathways [51] , [52] , [55] . Here we show that in addition to defective antigen presentation by CD11b + DCs, HDM-challenged DNA-PKcs fl/fl ; CD11c -Cre mice had an increase in BALF levels of IL-10 and BMDCs from DNA-PKcs fl/fl ; CD11c-Cre mice secreted increased amounts of IL-10 in response to HDM. IL-10 production by BDMCs from WT mice was increased following Akt inhibition, which is consistent with a ROS-activated pathway in HDM-stimulated DCs that signals via DNA-PK and Akt to attenuate IL-10 production. Thus, increases in IL-10 production may also contribute to the reduced allergic sensitization and Th2-type inflammation in HDM-challenged DNA-PKcs fl/fl ; CD11c Cre mice. We also assessed whether pharmacological inhibition of DNA-PK might represent an effective therapeutic approach to attenuate the manifestations of HDM-mediated allergic asthma. NU7441 (8-diebenzothiopen-4-yl-2-morpholin-4-yl-chromen-4-one) is a highly potent and selective ATP-competitive inhibitor of DNA-PK (IC 50 =0.014 uM) that was initially identified by screening of a chromenone library [56] . NU7441 was developed as an anticancer agent on the basis of its ability to potentiate cell death mediated by chemotherapy- and radiation therapy-induced DSBs [57] . Here we show that pharmacological inhibition of DNA-PK with NU7441 attenuated the induction of HDM-induced allergic sensitization, as well as Th2 effector cytokine production, airway inflammation, mucous cell metaplasia and AHR. In addition, initiation of NU7441 treatment after T-cell priming had already occurred similarly reduced HDM-induced airway inflammation, mucous cell metaplasia and AHR. Thus, we propose the concept of targeting DNA-PK with small molecule pharmacological inhibitors that might be developed as a novel treatment approach for patients with allergic asthma. To avoid systemic effects, site-directed delivery of a DNA-PK inhibitor directly to the lungs via inhalation would likely represent the preferred method of administration. To the best of our knowledge, our report is the first to describe a role for DNA-PK in modulating DC function in the pathogenesis of Th2 immune responses to HDM in experimental allergen-induced asthma. We propose that this is a novel and unexpected function for DNA-PK in DCs, as the adoptive transfer of CD4 + T cells into Prkdc scid mice has induced or enhanced disease in experimental murine models of colitis, skin allograft rejection and Pneumocystis pneumonia, which suggests that DC function in these settings is sufficient to mediate disease [58] , [59] , [60] . Additional studies will therefore be required to elucidate the dichotomy in DC function between experimental allergic asthma and other CD4 + T-cell-mediated disorders. In summary, we have identified a novel function for DNA-PK in DCs where it is required for effective antigen presentation and the subsequent induction of allergic sensitization and Th2 immunity to HDM in the airway. We show that HDM induces phosphorylation and activation of DNA-PK via a ROS-dependent pathway and that ROS production by DCs is DNA-PK-dependent. Furthermore, we demonstrate that pharmacological inhibition of DNA-PK with NU7441 attenuates the cardinal manifestations of experimental HDM-induced asthma, including allergic sensitization, Th2-mediated airway inflammation, mucous cell metaplasia and AHR. This identifies DNA-PK as a potential therapeutic target in asthma and can serve as the basis for the future development of DNA-PK inhibitors as a new treatment approach for patients with asthma. Reagents NU7441 was from Tocris Bioscience (Bristol, UK). DPI and NAC were from Calbiochem (EMD Millipore, Billerica, MA, USA). HDM ( Dermatophagoides pteronyssinus ) extract was purchased from Greer Laboratories, Lenoir, NC, USA as a freeze-dried preparation (Item no. B82). The Akt inhibitors GDC0068 and MK2206 were from Cellagen Technology (San Jose, CA, USA) and Selleckchem (Houston, TX, USA), respectively. Quantikine ELISA kits for measurement of cytokines and chemokines were from R&D Systems (Minneapolis, MN, USA). Mice BALB/c, C57BL/6, Prkdc scid (CBySmn.CB17- Prkdc scid ), DO11.10 TCR (C.Cg-Tg(DO11.10)10Dlo), which express a transgenic MHCII-restricted TCR that binds the OVA peptide antigen, OVA 323–339 (ref. 24 ), and Cd11c -Cre (B6.Cg-Tg(Itgax-cre)1-1Reiz/J) mice were purchased from The Jackson Laboratories (Bar Harbor, MA, USA). Six- to eight-week-old female mice were utilized for experiments. Murine experimental protocols were approved by the Animal Care and Use Committee of the National Heart, Lung, and Blood Institute, Bethesda, MD, USA. To generate the DNA-PKcs fl/fl mouse, a LoxP site was inserted between exons 81 and 82 of a 3.6-kb Hind III–SacI fragment of the mouse Prkdc gene in pBluescript II SK to give p1227 by using a Quikchange kit from Agilent Technologies (Santa Clara, CA, USA) and oligo PKKpnLoxP2 (5′- CCTCCCAAGTGCTGGGATTAGGTACCATAACTTCGTATAATGTATGCTATACGAAGTTATAAGGCGTGCACTACCACTGC -3′). The insert resulting from the SacI digestion of p1227 was transferred into a SacI-digested plasmid pBSK-H3 that contained a 7.5-kb HindIII fragment of mouse Prkdc in pBluescript II SK, to generate plasmid p1228. A SalI–NotI fragment encoding FRT-Neo-FRT-Loxp from plasmid pL451 ( http://ncifrederick.cancer.gov/research/brb/productDataSheets/recombineering/plasmid.aspx#PL451 ) was cloned between Prkdc exons 83 and 84 by PacI digestion of plasmid p1228 (ref. 61 ). The final construct was linearized by digestion with NotI for electroporation into the v6.5 mouse ES cell line (a 129 and C57BL/6J F1 hybrid ES cell line) [62] . Electroporated ES cells were grown in culture media containing both G418, for positive selection, and ganciclovir for negative selection. ES cell clones resistant to G418 and ganciclovir were screened for targeted insertion by Southern blotting. ES cell clones with correct homologous recombination were injected into blastocyst-stage embryos, which were then transferred to the uteri of surrogate mothers. F0 generation mice born from the injected embryos are chimeras composed of genetic contributions from both the modified ES cells and the recipient embryos. To obtain mouse lines that carry the gene-targeted mutation, we bred the chimeras to transmit the ES cell genetic component through the germ line. Once germ line transmission was established, mice were back-crossed to C57BL/6J mice for at least 10 generations. DNA-PKcs fl/fl mice were then bred with CD11c -Cre mice to generate DNA-PKcs fl/fl ; CD11c -Cre mice that were homozygous at each allele. Both male and female DNA-PKcs fl/fl and DNA-PKcs fl/fl ; CD11c -Cre mice that were 6–8 weeks old were utilized for experiments. Southern blotting An exon 79 probe labelled with 32 P by nick translation was used for Southern blotting to identify a 10-kb band for the modified Prkdc allele when genomic DNA was digested with EcoRI, while an exon 86 probe identified an 8.4-kb band when genomic DNA was digested with BamHI. Genotyping and genomic sequencing The following oligonucleotides, which flank the 5′ LoxP of the targeting construct, were used as primers for PCR genotyping reactions; PKEx81f (5′- CTGGAGCCTATGTGCTAATGTACAG -3′) and PKEx82r (5′- CTGTTTCTGTACGGTTAGCTCGGCTG -3′). Genomic DNA was isolated from flow-sorted cells using a DNAeasy kit (Qiagen) and PCR was performed using HotStar Taq (Qiagen). Amplification products were separated on 2% agarose gels that were stained with ethidium bromide to visualize a 646-bp band. Genomic DNA from flow-sorted cells was amplified with PCR using the following primers: NotpKEX81f (5′- GGGCGGCCGCCTGGAGCCTATGTGCTAATGTACAG -3′) and NotminusLoxPr (5′- GGGCGGCCGCGTGTCAGGTTTCATAACAATGCC -3′). Overlapping DNA sequences were obtained with PCR using the following primer pairs: PKseq30f (5′- GTTCTCTTGAGAGCTCTGGTCCG -3′) and PK Ex84seqr (5′- GGCATCAACTCAGGGACTGGAAG -3′), as well as NotpKEX81f and pKseq30r (5′- CGGACCAGAGCTCTCAAGAGAAC -3′). The amplified DNA was cloned and sequenced. Quantitative reverse transcription (qRT–PCR) RNA was isolated from the same flow-sorted cells using trizol reagent (Life Technologies, Grand Island, NY, USA) and cDNA was generated using a High Capacity RNA-to-cDNA kit (Applied Biosystems). The cDNA was pre-amplified by PCR using oligos PKEx81f and PKEx83r (5′- CTGAGTAGCTGATCCAAACGC -3′) and HotStar Taq. qRT–PCR was performed in triplicate for each sample using a Taqman gene expression assay (Mm01342966_g1, Life Technologies) that spans the junction between exons 82 and 83 of mouse DNA-PKcs and was normalized to 18S RNA. The assay was repeated three times. Derivation of DCs from monocytes and bone marrow cells Elutriated human monocytes, which had been obtained from normal volunteers who had provided informed consent to participate in an institutional review board-approved protocol (01-CC-0168), were provided by the Department of Transfusion Medicine, NIH Clinical Center. Monocytes were cultured in RPMI-1640 medium containing 10% fetal bovine serum (FBS), L-glutamine (2 mM), penicillin (100 U ml −1 ), streptomycin (100 μg ml −1 ; Gibco/Life Technologies), human recombinant granulocyte–macrophage colony-stimulating factor (150 ng ml −1 ) and IL-4 (25 ng ml −1 ; BioLegend, San Diego, CA, USA) in 10 cm petri dishes (BD Biosciences, San Jose, CA, USA) for 7 days before experimentation to induce the differentiation of moDCs [63] . CD11c + /HLA-DR + /CD14 − human moDCs were analysed with flow cytometry using the following antibodies, CD11c-APC, HLA-DR-PerCP/Cy5.5, CD14-Alexa Fluor 488, CD40-Alexa Fluor 647, CD80-Brilliant Violet 605 and CD86-PE, all from Biolegend. Cell viability was assessed using Fixable Viability Dye eFluor 450 (eBioscience, San Diego, CA). Bone marrow cells were isolated from the leg bones of euthanized WT and Prkdc scid mice and cultured at a density of 2 × 10 6 cells ml −1 in RPMI 1,640 medium containing 10% heat-inactivated FCS, penicillin (100 U ml −1 ), streptomycin (100 μg ml −1 ), L-glutamine (2 mM), 2-mercaptoethanol (50 μM) and recombinant mouse granulocyte–macrophage colony-stimulating factor (20 ng ml −1 ). Cultures were supplemented with an equal volume of medium on day 3 and 50% of the medium was replaced on day 6. Non-adherent cells were collected on day 8 and viable CD11c + BMDCs were sorted with flow cytometry using a CD11c-APC-Cy7 antibody from BD Biosciences. BMDCs were analysed with flow cytometry using the following antibodies, CD11c-APC-eFluor 780, MHCII-PE-Cy7, CD40-APC, CD80-Cy5, CD86-eFluor 605 NC and Fixable Viability Dye eFluor 450, all from eBioscience. Western blot analysis Human moDCs were lysed in RIPA buffer and 100 μg of protein that had been separated by SDS–PAGE using 4–20% Tris-Glycine gels (Lonza, Walkersville, MD, USA) was transferred to nitrocellulose membranes (GE Healthcare Life Sciences, Pittsburgh, PA, USA). Membranes were reacted with antibodies (1:1,000 dilution) directed against phospho-DNA-PKcs (Ser2056; Abcam, Cambridge, MA, USA); DNA-PKcs (Thermo Scientific, Pittsburgh, PA); phospho-Akt (Ser473), phospho-Akt (Thr308), Akt (Cell Signaling Technology, Danvers, MA); and β-actin (Santa Cruz Biotechnology, Santa Cruz, CA). Blots were stripped using Restore Western Blot Stripping Buffer (Thermo Scientific). Measurement of intracellular ROS Cultures of human moDCs and BMDCs from WT C57BL6 and Prkdc SCID mice were incubated with 2 μM of the redox-sensitive probe, CM-H 2 DCFDA, (5-(and-6)-chloromethyl-2′,7′-dichlorodihydrofluorescein diacetate, acetyl ester; Molecular Probes, Life Technologies) for 30 min at 37 °C. Oxidation of the CM-H 2 DCFDA probe with ROS produces a stable fluorescent adduct that was detected by an increase in fluorescence in the fluorescein channel. Levels of intracellular ROS generated in response to treatment with HDM (100 μg ml −1 ) for 1 h were quantified by subtracting the background MFI of the nonfluorescent sample (negative control) from the measured MFI values of fluorescent samples in the flow cytometry analysis. OVA-induced T-cell proliferation and Th2 cytokine production BMDCs from WT BALB/c and Prkdc scid mice were pulsed overnight with 1 μg ml −1 of OVA 323–339 peptide (AnaSpec, Fremont, CA, USA) or PBS as a control and viable CD11c + cells were isolated by flow sorting using an anti-mouse CD11c-APC-Cy7 antibody (BD Biosciences). Naive CD4 + T cells were purified from the spleens of DO11.10 TCR mice by flow sorting using an anti-mouse CD4-eFluor 650NC antibody (eBioscience) and were labelled with 5 μM CFDA-SE (carboxyfluorescein diacetate succinimidyl ester; Cayman Chemical, MI, USA) for 30 min. Overall, 1 × 10 5 OVA peptide-specific CD4 + T cells were co-cultured with 2 × 10 4 CD11c + BMDCs in 96-well plates for 4 days, and T-cell proliferation was quantified with flow cytometry using the CSFE dye dilution method. The ‘Proliferation Ratio’ is the MFI of CSFE-SE from OVA 323–339 peptide-pulsed CD11c + BMDCs divided by the MFI of CSFE-SE from PBS-pulsed CD11c + BMDCs. The quantity of IL-4, IL-5 and IL-13 released into the culture medium after 4 days was measured using ELISA. For experiments assessing priming with full-length OVA, female BALB/c mice (6–8 weeks old) received intraperitoneal injections of OVA (Sigma-Aldrich, St Louis, MO, USA) emulsified in 0.2 ml of sterile PBS containing 2 mg of aluminium hydroxide (Sigma-Aldrich) on days 0 and 7. Overall, 10 5 splenic CD4 + T cells were purified by flow sorting on day 10, co-cultured with BMDCs from WT and Prkdc scid mice at a 5:1 ratio in a medium containing full-length OVA (1 μg ml −1 ) for 4 days in 96-well plates, and the quantity of cytokines released into the culture medium was measured with ELISA. HDM sensitization and challenge models (1) Adoptive transfer of CD11c + BMDCs from Prkdc scid mice. CD11c + BMDCs that had been isolated from WT and Prkdc scid mice using flow cytometry were pulsed with HDM (100 μg ml −1 ) or PBS for 16 h. Overall, 5 × 10 4 viable CD11c + BMDCs were adoptively transferred in 20 μl of PBS via intranasal administration on day 0 to recipient WT C57BL/6 mice. Recipient mice received daily intranasal HDM challenges (25 μg) on days 11 through 13 and end points were analysed on day 15. The HDM extracts contained between 29.1 and 50 endotoxin units mg −1 of HDM protein, which resulted in 73–125 pg of lipopolysaccharide being administered with each 25 μg dose of HDM. (2) Adoptive transfer of CD11c + BMDCs treated with NU7441 or GDC0068. CD11c + BMDCs that had been isolated from WT BALB/c mice using flow cytometry were pulsed with HDM (100 μg ml −1 ) in the presence or absence of NU7441 (0.5 μM), GDC0068 (1 μM) or PBS for 16 h. Overall, 5 × 10 4 viable CD11c + BMDCs were adoptively transferred in 20 μl of PBS via intranasal administration on day 0 to recipient WT BALB/c mice. Recipient mice received daily intranasal HDM challenges (25 μg) on days 11 through 13 and end points were analysed on day 15. (3) Intranasal sensitization and challenge of DNA-PKcs fl/fl and DNA-PKcs fl/fl CD11c Cre mice. DNA-PKcs fl/fl and DNA-PKcs fl/fl CD11c Cre mice were sensitized and challenged via daily intranasal administration of 25 μg of HDM or PBS, both in a volume of 10 μl, 5 days a week, for 6 weeks. (4) Adoptive transfer of CD11b + DCs isolated from MLNs of HDM-pulsed DNA-PKcs fl/fl and DNA-PKcs fl/fl ; Cd11c-Cre mice. DCs from DNA-PKcs fl/fl and DNA-PKcs fl/fl ; Cd11c -Cre mice were loaded in vivo with HDM allergen by intranasal instillation of HDM extract (100 μg), or saline as a control, using a modification of a previously described protocol [29] . After 4 days, mice were killed, MLNs were removed and CD11c + /CD11b + /SiglecF − /MHCII + DCs were isolated with flow cytometry using a FACS-ARIA II flow sorter (BD Biosciences) and the following antibodies: CD11c-APC-Cy7 and SiglecF Alexa Fluor 647, both from BD Biosciences, CD11b-PerCP-Cy5.5 (eBioscience) and MHCII-PE-Cy7 from Biolegend. Overall, 2.5 × 10 4 CD11c + /CD11b + /SiglecF − /MHCII + DCs were adoptively transferred to WT C57BL/6 recipient mice by intranasal administration in a volume of 20 μl. All recipient mice received daily intranasal HDM challenges (25 μg) on days 9 through 14 and end points were analysed on day 15. (5) Oral administration of NU7441. WT BALB/c were sensitized and challenged by daily intranasal administration of HDM (25 μg) or PBS, both in a volume of 10 μl, 5 days a week for 4 weeks. Mice were fed chow that contained 0, 0.6 or 0.9% NU7441 (TestDiet, St Louis, MO, USA) throughout the 4-week study period. For experiments assessing the effect of NU7441 administration only during the HDM challenge phase, WT BALB/c mice were sensitized by intraperitoneal injection of HDM (100 μg) emulsified in 200 μl of PBS containing 3 mg of aluminium hydroxide (Sigma-Aldrich) on days 0 and 4. Mice were challenged by intranasal administration of HDM (100 μg) in a volume of 40 μl on days 8, 10 and 12 and end points were analysed on day 14. Mice were fed chow that contained 0.9% NU7441 starting day 8, coincident with the start of the challenge phase of the protocol. Control mice were both sensitized and challenged with saline and were fed regular chow. Analysis of BALF and lung histopathology Bronchoalveolar lavage was performed three times with 0.5 ml of PBS. Red blood cells were lysed with ACK buffer for 2 min at 4 o C and cells were re-suspended in RPMI-1640 medium with 10% FBS. BALF cell counts were performed using a hemocytometer, and differential cell counts were performed on Diff-Quik-stained cytospin slides (Siemens, Deerfield, IL, USA). For histological analysis, lungs were inflated with 10% formalin to a pressure of 25 cm H 2 0, fixed in 10% formalin for 24 h, dehydrated through gradient ethanol, embedded in paraffin, sagittal sections cut to a thickness of 5 μm and stained with haematoxylin and eosin or periodic acid Schiff (PAS). Quantification of mucous cell metaplasia was performed by analysing all the airways present (large (conducting), medium (central) and small (distal)) within each representative lung section. The number of airways that contained PAS-positive cells was counted and mucous cell metaplasia is presented as the percentage of airways with PAS-positive cells. HDM-specific IgE Plates were coated overnight with 0.01% HDM in PBS and blocked with 1% BSA in PBS before the addition of serum samples that had been diluted 1:10 in blocking buffer and standards for 1 h. Plates were washed 6 × with PBS containing 0.05% Tween‐20 before incubation with biotinylated anti-mouse IgE (Pharmingen, San Jose, CA, USA) at a concentration of 2 μg ml −1 for 1 h. Plates were washed an additional six times, streptavidin-HRP (R&D Systems) was added for 30 min and the amount of bound HDM-specific antibody was determined using TMB substrate. Re-stimulation of ex vivo cultures of MLN cells with HDM Single-cell suspensions from MLNs were cultured at a density 0.2 × 10 6 cells ml −1 in round-bottom 96-well plates and pulsed with HDM (100 μg ml −1 ) for 72 h at 37 °C in RPMI medium containing 10% FBS. In selected experiments, cells were also treated with NU7441 (0.5 μM). Flow cytometry For genotyping of DNA-PKcs fl/fl and DNA-PKcs fl/fl ; CD11c -Cre mice, CD11c + /MHCII + /SiglecF − DCs were isolated from spleens with flow sorting using a FACS-ARIA II flow cytometer (BD Biosciences) and with the following antibodies: CD11c-APC-Cy7, MHCII-PE-Cy7 and SiglecF-AF647, all from BD Biosciences. Lung cells were isolated by enzymatic digestion using liberase (Roche, Indianapolis, IN, USA), 100 μg ml −1 and DNase I (Sigma-Aldrich), 0.2 mg ml −1 , in a volume of 1–2 ml per lung at 37 °C for 25 min with agitation. Cells from the digested lungs were incubated with anti-CD16/CD32 antibodies (clone 2.4G2; Pharmingen/BD Biosciences) to block Fcγ III/II receptors before surface staining. Lung alveolar type II epithelial cells were isolated as CD45 − /CD11c − /EpCAM + cells using the following antibodies: CD11c-APC-Cy7 and EpCAM-PE from BD Biosciences and CD45R-650NC from eBioscience [64] . CD3 + T cells and CD19 + B cells present in the lungs and spleens of WT C57BL/6, DNA-PKcs fl/fl and DNA-PKcs fl/fl ; Cd11c -Cre mice were analysed using CD3-APC and CD19-APC-Cy7, both from Biolegend, while the Fixable Viability Dye eFluor 450 was from eBioscience. CD11c + /MHC hi /SSC lo DCs present in lungs and MLNs of HDM-challenged DNA-PKcs fl/fl and DNA-PKcs fl/fl ; Cd11c -Cre mice were analysed using the following anti-mouse antibodies: CD252 (OX-40L)-PE, CD40-APC, CD80-PE-Cy5 and CD86-eFluor 605 NC, all from eBioscience. CD11b + DCs were identified using a CD11b-PerCP-Cy5.5 antibody (eBioscience), while TLR4 and TLR5 expression on CD11c + /MHCII hi /SSC lo /CD11b + DCs were analysed using TLR4-APC from Biolegend and TLR5-PE antibodies from Novus Biologics (Littleton, CO, USA). Tregs were analysed using CD3-APC, CD4-eFluor 650NC and CD25-PE-Cy7, all from eBiosciences. For quantification of intracellular Foxp3, cells were fixed and permeabilized with Foxp3 staining buffer and reacted with a Foxp3-PE antibody, both from eBioscience. All antibodies were utilized at a concentration of 0.5–1 μg ml −1 . Data were acquired on a LSR-II (BD Biosciences) equipped with 407, 488, 532 and 633 LASER lines using the DIVA 6.1.2 software and analysed with the Flow Jo software version 9.6.1 (Treestar, San Carlos, CA, USA). Cellular debris was excluded using a forward light scatter/side scatter plot. For analysis of intracellular cytokines, 1 × 10 6 BAL cells ml −1 were suspended in RPMI-1640 supplemented with 10% FBS, L -glutamine (2 mM), penicillin (100 U ml −1 ) and streptomycin (100 μg ml −1 ), cultured in 24-well flat-bottom plates and stimulated with phorbol myristate acetate (50 ng ml −1 ), ionomycin (500 ng ml −1 ) and brefeldin A (3 μg ml −1 ; eBiosciences) for 4 h at 37 °C. Cells were washed with PBS, re-suspended in Flow Cytometry Staining Buffer (eBiosciences) containing 10% mouse serum (Jackson ImmunoResearch Inc., West Grove, PA, USA) and reacted with 5 μg ml −1 of rat anti-mouse CD3-APC-Cy7 and CD4-eFluor 650NC for 30 min, followed by two additional washes. Cells were treated with DNase I (60 μg ml −1 ) for 15 min at 37 °C, washed and re-suspended in 300 μl of permeabilization buffer containing 1% anti-mouse CD16/CD32 for 20 min. Cells were then reacted with rat anti-mouse IL-5-PE, IL-13-APC and IL-17-PE-Cy7 (eBiosciences) for 45 min at 4 °C. Cells were washed twice with permeabilization buffer, re-suspended in PBS containing 1% paraformaldehyde and viable CD3 +/ CD4 + T cells that expressed IL-5, IL-13 or IL-17 were quantified using the LSR-II using FMO (fluorescence minus one) as controls using Flow Jo analysis software. Analysis of DC migration to MLNs HDM (50 μg) that had been labelled with the Alexa Fluor 647 (AF647) Protein Labeling Kit (Molecular Probes, Life Technologies) was administered in 80 μl of PBS by i.t. instillation to DNA-PKcs fl/fl and DNA-PKcs fl/fl CD11c Cre mice [29] . Lungs and MLNs were harvested after 72 h and the number of CD11c + /MHCII hi /SSC lo /CD11b + /HDM + DCs were quantified with flow cytometry. Airway hyper-responsiveness Following cannulation of the trachea with a 19-gauge beveled metal catheter, airway resistance to increasing concentrations of methacholine (0–10 mg ml −1 ) was directly measured in mechanically ventilated mice using an Elan RC Fine Pointe system (Buxco, Wilmington, NC, USA) and average values are presented as cm H 2 O per ml s −1 . Statistics Data were analysed using Graph Pad Prism version 5.0a and are presented as mean±s.e.m. A one-way analysis of variance with Bonferroni’s or Sidak’s multiple comparison test, a Mann–Whitney test or an unpaired t -test were used for the analyses. A P value<0.05 was considered significant. How to cite this article: Mishra, A. et al . Dendritic cells induce Th2-mediated airway inflammatory responses to house dust mite via DNA-dependent protein kinase. Nat. Commun. 6:6224 doi: 10.1038/ncomms7224 (2015).